HSP90 regulates DNA repair via the interaction between XRCC1 and DNA polymerase β Cellular DNA repair processes are crucial to maintain genome stability and integrity. In DNA base excision repair, a tight heterodimer complex formed by DNA polymerase β (Polβ) and XRCC1 is thought to facilitate repair by recruiting Polβ to DNA damage sites. Here we show that disruption of the complex does not impact DNA damage response or DNA repair. Instead, the heterodimer formation is required to prevent ubiquitylation and degradation of Polβ. In contrast, the stability of the XRCC1 monomer is protected from CHIP-mediated ubiquitylation by interaction with the binding partner HSP90. In response to cellular proliferation and DNA damage, proteasome and HSP90-mediated regulation of Polβ and XRCC1 alters the DNA repair complex architecture. We propose that protein stability, mediated by DNA repair protein complex formation, functions as a regulatory mechanism for DNA repair pathway choice in the context of cell cycle progression and genome surveillance. Genome stability requires efficient DNA repair and DNA damage response protein complexes. Base excision repair (BER) is essential to provide nuclear and mitochondrial genome stability by repairing greater than 20,000 spontaneous base lesions per cell per day [1] . As with gross genomic changes such as DNA double-strand breaks, DNA base damage can also lead to genome instability and elevated cancer incidence if left unrepaired [2] . Base damage is repaired by proteins of the BER machinery via numerous sub-pathways that vary depending on the lesion type and the size of the repair patch [3] , [4] , [5] . Upon damage, poly(ADP-ribose)polymerase 1 (PARP1) activation triggers BER protein recruitment to facilitate short-patch or long-patch BER via DNA polymerase β (Polβ)-dependent or Polβ-independent mechanisms [3] , [4] , [6] , [7] . An essential component of BER and other DNA repair complexes is the scaffold protein XRCC1 (ref. 8 ). Interestingly, XRCC1 has no enzymatic activity and it is thought that its sole function is to promote DNA repair protein recruitment to the site of DNA damage. XRCC1 complexes with numerous BER proteins including DNA ligase III, Polβ, aprataxin and PARP1, among others [3] . In response to PARP1 activation, XRCC1 recruitment is thought to promote the formation of secondary BER protein complexes via interaction with these downstream factors to complete repair [4] . A paradigm repair protein complex is represented by the heterodimer of Polβ and XRCC1 (ref. 9 ). The two proteins (Polβ and XRCC1) form a tight-binding complex suggested to facilitate recruitment of Polβ to the site of repair following PARP1 activation [10] . However, mouse models for XRCC1 and Polβ have drastically different phenotypes, pointing to independent yet crucial roles for both partners of the complex. Mice lacking Polβ die just after birth [11] , whereas XRCC1 knockout (KO) mice do not develop beyond an early stage of embryogenesis, embryonic day 6.5 (ref. 12 ). This early developmental failure and lethality underlines the crucial role for BER in embryogenesis, development and genome stability. Importantly, whereas both proteins may play a significant role together as a complex, these mouse models suggest that Polβ and XRCC1 may have separate roles in mammalian development and cellular function. This study was initiated to reveal the function and significance of conserved DNA repair protein interactions exemplified by the Polβ/XRCC1 heterodimer. Guided by the structure of the heterodimer comprised of the carboxy-terminal domain of rat-Polβ (residues 142–335) and the amino-terminal domain of human XRCC1 (residues 1–151) [9] , we developed separation-of-function mutants of Polβ that retain the polymerase activity but are unable to form a heterodimer with XRCC1. Surprisingly, we find that the interaction between Polβ and XRCC1 is not required for the in vivo function of Polβ. However, our study has revealed the primary function of this evolutionarily conserved interaction interface is to maintain protein stability of each monomer: Polβ and XRCC1. Once released from XRCC1, we find that free Polβ is ubiquitylated on two lysines in the C-terminal domain and degraded by the proteasome independent of the E3 ligases CHIP or MULE. Conversely, XRCC1, not bound to Polβ, forms a complex with HSP90 that stabilizes XRCC1 protein levels. Knockdown or inactivation of HSP90 initiates ubiquitylation and degradation of XRCC1, mediated by CHIP. We provide evidence that the dynamic interaction of Polβ, XRCC1 and HSP90, via the two heterodimers Polβ/XRCC1 and XRCC1/HSP90, is regulated by the cell cycle and in response to DNA damage. We suggest that the dynamic interchange between the Polβ/XRCC1 and XRCC1/HSP90 heterodimers regulates DNA repair pathway choice. In summary, this study reveals an unexpected function of the evolutionarily conserved interaction domain between two DNA repair proteins. Challenging its recruitment function, here we report that the primary role for the scaffold protein XRCC1, together with HSP90, is to govern stability of its protein complex partners. Polβ V303 loop is essential for the interaction with XRCC1 DNA polymerase β (Polβ) and XRCC1 form a BER sub-complex via the C-terminal domain of Polβ and the N-terminal domain of XRCC1. A prominent feature of the interface is the Polβ V303 loop, comprised of amino-acid residues P300 to E309 and a hydrophobic pocket on XRCC1, spanning amino-acid residues F67 to V86, but may also include both β-strands D and E of XRCC1 (refs 13 , 14 ). Guided by the crystal structure of the rat-Polβ(C-term)/human-XRCC1(N-term) complex [9] , we identified several potential residues in the human-Polβ/human-XRCC1 interface region critical for complex formation. We mutated amino-acid residues in the Polβ V303 loop (L301, V303 and V306) to define the specific residues essential for Polβ/XRCC1 complex formation ( Fig. 1a ). To determine whether these V303 loop mutants of Polβ disrupt the Polβ/XRCC1 heterodimeric complex, stable LN428 cell lines were developed by lentiviral-mediated transduction to express Polβ (Flag-Polβ(WT)) or the V303 loop mutants, with modifications in amino-acid residues L301, V303 and/or V306. The relative expression level of Polβ and the V303 loop mutants in LN428 cells was examined and shown (see Supplementary Fig. 1B and below). The targeted amino-acid residues are depicted by the highlighted spheres in the structure shown ( Fig. 1a ). The presence of the Polβ/XRCC1 complex in these cells was probed by immunoprecipitation (IP) of the lentiviral-expressed Flag-Polβ transgene via the N-terminal Flag epitope tag and probing for XRCC1 by immunoblot ( Fig. 1b ). Mutating residues L301 or V306 individually or together had only a minimal impact, whereas mutating residue 303 (V303R) reduced the Polβ/XRCC1 complex formation by 90%. Altering both the L301 and V303 residues (L301R/V303R) resulted in a 99% loss ( Fig. 1b ; Supplementary Fig. S1A ). Finally, altering all three residues identified by the crystal structure analysis ( Fig. 1a ; Polβ(L301R/V303R/V306R), referred to herein as Flag-Polβ(TM)) completely abolished the interaction between Polβ and XRCC1 as determined by IP of either Polβ or XRCC1 ( Fig. 1b,c ; Supplementary Fig. 1A ). Analysis of the IP complexes by mass spectrometry also confirms the loss of XRCC1 binding to Flag-Polβ(TM) ( Supplementary Fig. 8 ). Note the equivalent amount of Polβ proteins in the immunoprecipitation clearly demonstrates the loss of binding between Flag-Polβ(TM) and XRCC1. These data establish that the Polβ V303 loop, in particular the V303 residue, forms an essential complex-formation interface with XRCC1. 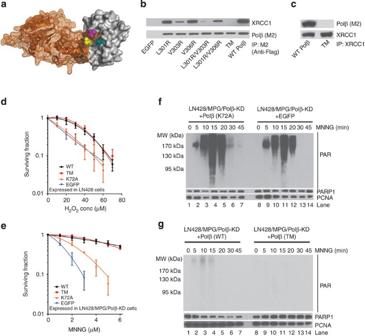Figure 1: Complex formation between DNA polymerase β and XRCC1 is not essential for the cellular response to DNA damage. (a) Structure (pdb3lqc) depicting oxidized XRCC1 (residues 1–151) bound to Polβ (residues 142–335)9. The image is a cartoon rendition of the palm and thumb domains of Polβ in orange with a mesh illustrating the surface of the structure and a space-filling rendition of the oxidized form of XRCC1 in grey with a solid illustrating the surface of the structure. Amino acids L301 (yellow), V303 (cyan) and V306 (magenta) are shown using a space-filling rendering. The images were generated using PyMOL (Molecular Graphics System, Version 1.2r3pre; Schrödinger, LLC). (b) Stable LN428 cell lines expressing Flag-Polβ(WT) or the V303 loop mutants were probed for Polβ/XRCC1 complex formation by IP of the lentiviral-expressed Flag-Polβ transgene via the N-terminal Flag epitope tag and probing for XRCC1 and Flag-Polβ by immunoblot (see alsoSupplementary Fig. 9). (c) Stable LN428 cell lines expressing Flag-Polβ(WT) or Flag-Polβ(TM) were probed for Polβ/XRCC1 complex formation by IP of XRCC1 (XRCC1-Ab) and probing for XRCC1 and Polβ by immunoblot. (d) Cell viability of LN428 cells expressing Flag-Polβ(WT), Flag-Polβ(TM), Flag-Polβ(K72A) or EGFP (as indicated) after H2O2treatment, as measured by the long-term assay. Plots show the relative surviving fraction as compared with untreated (control) cells. Means are calculated from triplicate values in each experiment. Results indicate the mean±s.d. of three independent experiments. (e) Cell viability of LN428/MPG/Polβ-KD cells expressing Flag-Polβ(WT), Flag-Polβ(TM), Flag-Polβ(K72A) or EGFP (as indicated) after MNNG treatment, as measured by the MTS assay 48 h after exposure. Plots show the relative surviving fraction as compared with untreated (control) cells. Results indicate the mean±s.d. of three independent experiments. (f) Immunoblot of PAR to determine activation of PARP after exposure to MNNG (5 μM) for the time indicated for LN428/MPG/Polβ-KD cells expressing Flag-Polβ(K72A) (left panel) or EGFP (right panel). PARP1 and PCNA protein expression levels are also shown as loading controls. (g) Immunoblot of PAR to determine activation of PARP after exposure to MNNG (5 μM) for the time indicated for LN428/MPG/Polβ-KD cells expressing Flag-Polβ(WT) (left panel) or Flag-Polβ(TM) (right panel). PARP1 and PCNA protein expression levels are also shown as loading controls. Figure 1: Complex formation between DNA polymerase β and XRCC1 is not essential for the cellular response to DNA damage. ( a ) Structure (pdb3lqc) depicting oxidized XRCC1 (residues 1–151) bound to Polβ (residues 142–335) [9] . The image is a cartoon rendition of the palm and thumb domains of Polβ in orange with a mesh illustrating the surface of the structure and a space-filling rendition of the oxidized form of XRCC1 in grey with a solid illustrating the surface of the structure. Amino acids L301 (yellow), V303 (cyan) and V306 (magenta) are shown using a space-filling rendering. The images were generated using PyMOL (Molecular Graphics System, Version 1.2r3pre; Schrödinger, LLC). ( b ) Stable LN428 cell lines expressing Flag-Polβ(WT) or the V303 loop mutants were probed for Polβ/XRCC1 complex formation by IP of the lentiviral-expressed Flag-Polβ transgene via the N-terminal Flag epitope tag and probing for XRCC1 and Flag-Polβ by immunoblot (see also Supplementary Fig. 9 ). ( c ) Stable LN428 cell lines expressing Flag-Polβ(WT) or Flag-Polβ(TM) were probed for Polβ/XRCC1 complex formation by IP of XRCC1 (XRCC1-Ab) and probing for XRCC1 and Polβ by immunoblot. ( d ) Cell viability of LN428 cells expressing Flag-Polβ(WT), Flag-Polβ(TM), Flag-Polβ(K72A) or EGFP (as indicated) after H 2 O 2 treatment, as measured by the long-term assay. Plots show the relative surviving fraction as compared with untreated (control) cells. Means are calculated from triplicate values in each experiment. Results indicate the mean±s.d. of three independent experiments. ( e ) Cell viability of LN428/MPG/Polβ-KD cells expressing Flag-Polβ(WT), Flag-Polβ(TM), Flag-Polβ(K72A) or EGFP (as indicated) after MNNG treatment, as measured by the MTS assay 48 h after exposure. Plots show the relative surviving fraction as compared with untreated (control) cells. Results indicate the mean±s.d. of three independent experiments. ( f ) Immunoblot of PAR to determine activation of PARP after exposure to MNNG (5 μM) for the time indicated for LN428/MPG/Polβ-KD cells expressing Flag-Polβ(K72A) (left panel) or EGFP (right panel). PARP1 and PCNA protein expression levels are also shown as loading controls. ( g ) Immunoblot of PAR to determine activation of PARP after exposure to MNNG (5 μM) for the time indicated for LN428/MPG/Polβ-KD cells expressing Flag-Polβ(WT) (left panel) or Flag-Polβ(TM) (right panel). PARP1 and PCNA protein expression levels are also shown as loading controls. Full size image Polβ/XRCC1 complex is not essential for DNA damage response The interaction of XRCC1 with Polβ has been thought to be essential to complete repair. As a consequence, sensitivity to oxidative stress or alkylation damage is determined by BER efficiency [3] such as that defined by XRCC1 or Polβ proficiency. Since Flag-Polβ(TM) is completely devoid of the ability to interact with XRCC1, we used these constructs to determine whether the interaction of Polβ and XRCC1 is essential for the response to DNA damage in human cells. We used cells expressing Flag-Polβ(K72A), which inactivates the 5′dRP lyase activity of Polβ, or cells expressing EGFP as control cells [15] . Human LN428 glioma cells expressing Flag-Polβ(WT), Flag-Polβ(TM), Flag-Polβ(K72A) or EGFP (vector control) were treated with increasing concentrations of H 2 O 2 . Cell survival was determined using both short-term and long-term cell survival assays. Confirming a role for the 5′dRP lyase activity of Polβ in oxidative DNA damage-induced BER, the expression of Flag-Polβ(WT) confers resistance to H 2 O 2 , whereas expression of the 5′dRP lyase-defective mutant, Flag-Polβ(K72A), does not complement the Polβ deficiency ( Fig. 1d ; Supplementary Fig. 1C ). Importantly, no significant difference in cell survival was observed when comparing cells expressing Flag-Polβ(WT) or Flag-Polβ(TM) ( Fig. 1d ; Supplementary Fig. 1C ). Overall, we show that disruption of the Polβ/XRCC1 complex does not significantly impact H 2 O 2 -induced cytotoxicity in these cells. Similarly, we show that the ability for Polβ and XRCC1 to form a complex does not alter the cellular response to ionizing radiation (IR; Supplementary Fig. 1E ). The cellular response to alkyation damage is dependent on mismatch repair and BER, in particular, the expression of MPG, Polβ and XRCC1 (refs 16 , 17 , 18 , 19 ). Since LN428 cells are deficient in MPG expression, re-expression of N-methylpurine-DNA glycosylase (MPG) therefore promotes cellular dependence on BER capacity in response to alkylation damage. We therefore established LN428-derived cell lines that re-express MPG but are deficient in the expression of endogenous Polβ (LN428/MPG/Polβ-KD). Polβ knockdown results in the loss of more than 85% of endogenous Polβ as shown by the immunoblot ( Supplementary Fig. 7B ). Further, these cells were engineered, as above, for the expression of Flag-Polβ(WT), Flag-Polβ(TM), Flag-Polβ(K72A) or EGFP (vector control). As expected, cells expressing Flag-Polβ(K72A) or those deficient in the expression of Polβ (expressing EGFP) are very sensitive to N -methyl- N ′-nitro- N -nitrosoguanidine (MNNG)-induced DNA damage ( Fig. 1e ). However, similar to that seen in response to H 2 O 2 , cells expressing either Flag-Polβ(WT) or Flag-Polβ(TM) are equally resistant to MNNG ( Fig. 1e ). To further confirm the proficiency of Flag-Polβ(TM) to complement Polβ deficiency in response to alkylation damage, we next used T98G cells. T98G cells express elevated levels of MGMT ( Supplementary Fig. 1D ) and are therefore highly resistant to O 6 -MeG-induced cytotoxicity [17] , abrogating an involvement of mismatch repair for cell survival to alkylation damage and therefore allowing analysis by long-term cell survival assays. As above, we expressed Flag-Polβ(WT), Flag-Polβ(TM), Flag-Polβ(L301R/V303R) or EGFP (vector control) in T98G/MPG/Polβ-KD cells. As expected, cells deficient in the expression of Polβ are significantly more sensitive to MNNG ( Supplementary Fig. 1F ). Importantly, cells expressing Flag-Polβ(TM) or Flag-Polβ(L301R/V303R) can complement to the same extent as the wild-type (WT) protein. From this, we conclude, by analysis of multiple cell lines, that disruption of the Polβ/XRCC1 complex does not impact cytotoxicity induced by the alkylating agent MNNG. In response to DNA damage, PARP1 is activated and results in the formation of polymers of ADP-ribose, poly(ADP-ribose) (PAR). Defects in BER result in elevated PAR formation in response to DNA damage. As we have described earlier, a deficiency in Polβ will provoke elevated PARP1 activation in response to alkylation damage (as compared with cells expressing Polβ) [16] . We therefore evaluated the impact of disrupting the Polβ/XRCC1 interaction on DNA damage-induced PARP1 activation. PAR formation was compared in cells expressing Flag-Polβ(WT), Flag-Polβ(TM), Flag-Polβ(K72A) or EGFP (vector control) in response to MNNG exposure. As predicted, cells deficient in the expression of Polβ or those expressing the 5′dRP lyase mutant of Polβ, Flag-Polβ(K72A), yield robust PARP1 activation in response to MNNG treatment ( Fig. 1f ). However, in line with the cell survival assays shown in Fig. 1e , there is little or no PARP1 activation in cells expressing Flag-Polβ(WT) or Flag-Polβ(TM) after exposure to MNNG ( Fig. 1g ). These cell survival and PARP1 activation studies clearly establish that both Flag-Polβ(WT) and Flag-Polβ(TM) are functional proteins when expressed in cells and that the complex formed between Polβ and XRCC1 is not essential for the overall cellular response to DNA damage. Polβ is recruited to DNA damage sites via PARP1 activation Current models of nuclear BER suggest that PARP1 binds to APE1-induced DNA strand breaks during BER and initiates local PAR synthesis at the site of the lesion, facilitating BER protein recruitment to complete repair [3] , [20] , [21] . This model predicts that XRCC1 is subject to PAR-facilitated recruitment and that Polβ is recruited to the site via complex formation with XRCC1 (ref. 22 ). We therefore tested this model directly by evaluating whether the interaction between XRCC1 and Polβ is required for this recruitment. Recruitment of Polβ(WT) or Polβ(TM) to DNA repair foci was evaluated by two approaches: (i) loci-specific reactive oxygen species (ROS)-induced damage or (ii) 405 nm laser light-induced damage ( Fig. 2 ; Supplementary Fig. 2B ). In the first approach, we visualized BER protein recruitment in response to base damage using a recently developed KillerRed [23] , [24] system to produce local ROS-induced DNA damage within a single chromosomal location in the genome. In this system, ROS-induced DNA damage is generated on visible light exposure. Damage is localized to a tandem array of tetracycline response elements (TREs) [25] by binding of a KillerRed-tetR fusion protein ( Fig. 2a ), as we have recently reported [26] . This system provides a novel and effective approach to follow BER protein recruitment in response to ROS-mediated base damage [26] . We co-expressed KillerRed-tetR with copGFP, copGFP-Polβ(WT) or copGFP-Polβ(TM) in U2OS cells with the TRE arrays (U2OS-TRE; Fig. 2b ). Light exposure results in the appearance of a single, KillerRed foci ( Fig. 2b , middle panels). CopGFP-Polβ(WT) is recruited and co-localizes with KillerRed foci ( Fig. 2b ). Importantly, copGFP-Polβ(TM), similar to copGFP-Polβ(WT), also accumulates at the KillerRed-induced ROS damage site in the TRE, albeit at a lower level ( Fig. 2b,c ). 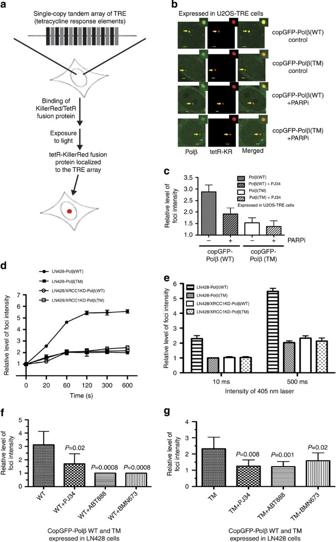Figure 2: DNA polymerase β is recruited to DNA damage sites via PARP1 activation independent of XRCC1 complex formation. (a) Diagram describing a U2OS cell line (U2OS-TRE) with an integrated single-copy tandem array of TREs and the light-induced localization of a KillerRed-tetR fusion protein to the TRE tandem array, mediated by the specific interaction between the TRE and the tetR protein, depicted by a red spot26. (b) Fluorescent images depicting DNA damage-induced foci of KillerRed-tetR and copGFP-Polβ(WT) or copGFP-Polβ(TM) expressed in U2OS-TRE cells after light exposure (10 min), as indicated in the figure. Arrows point to the foci induced by tetR-KR and copGFP-Polβ(WT) or copGFP-Polβ(TM) and after pre-incubation with the PARP inhibitor PJ34. Scale bar, 2 μm. (c) The relative intensity of copGFP-Polβ(WT) or copGFP-Polβ(TM) foci induced by KillerRed-mediated ROS23,26,69was quantified as shown. Results indicate the mean±s.d. of the analysis of 10 independent cells. (d) Kinetics of copGFP-Polβ(WT) or copGFP-Polβ(TM) recruitment to DNA damage sites. Cells were treated with a 405-nm laser (500 ms) and the images were obtained at the indicated times. The relative intensity of foci was then quantified. Results indicate mean±s.d. of three independent experiments. (e) The relative intensity of foci in cells treated with 10 ms or 500 ms 405 nm laser at 5 min was quantified. Results indicate mean±s.d. of three independent experiments. The representative images are shown inSupplementary Fig. 2B. (f,g) Suppression of (f) copGFP-Polβ(WT) or (g) copGFP-Polβ(TM) recruitment to DNA damage-induced foci by the PARP inhibitors ABT-888, PJ34 and BMN-673. Stable LN428 cells expressing copGFP-Polβ(WT) or/and copGFP-Polβ(TM) were pre-treated with PARP inhibitors (PJ34, 4 μM; ABT-888, 10 μM; or BMN-673, 5 μM) for 1 h or without PARP inhibitor treatment, then cells were exposed to the 405-nm laser (50 ms or 1,000 ms). Images of cells were obtained after 2 min laser treatment. Results indicate mean±s.d. of five to eight independent cells. A one-tailedt-test was used for the statistical analysis and thePvalue was determined comparing cells treated with the PARP inhibitors as compared with cells without PARP inhibitor treatment. Figure 2: DNA polymerase β is recruited to DNA damage sites via PARP1 activation independent of XRCC1 complex formation. ( a ) Diagram describing a U2OS cell line (U2OS-TRE) with an integrated single-copy tandem array of TREs and the light-induced localization of a KillerRed-tetR fusion protein to the TRE tandem array, mediated by the specific interaction between the TRE and the tetR protein, depicted by a red spot [26] . ( b ) Fluorescent images depicting DNA damage-induced foci of KillerRed-tetR and copGFP-Polβ(WT) or copGFP-Polβ(TM) expressed in U2OS-TRE cells after light exposure (10 min), as indicated in the figure. Arrows point to the foci induced by tetR-KR and copGFP-Polβ(WT) or copGFP-Polβ(TM) and after pre-incubation with the PARP inhibitor PJ34. Scale bar, 2 μm. ( c ) The relative intensity of copGFP-Polβ(WT) or copGFP-Polβ(TM) foci induced by KillerRed-mediated ROS [23] , [26] , [69] was quantified as shown. Results indicate the mean±s.d. of the analysis of 10 independent cells. ( d ) Kinetics of copGFP-Polβ(WT) or copGFP-Polβ(TM) recruitment to DNA damage sites. Cells were treated with a 405-nm laser (500 ms) and the images were obtained at the indicated times. The relative intensity of foci was then quantified. Results indicate mean±s.d. of three independent experiments. ( e ) The relative intensity of foci in cells treated with 10 ms or 500 ms 405 nm laser at 5 min was quantified. Results indicate mean±s.d. of three independent experiments. The representative images are shown in Supplementary Fig. 2B . ( f , g ) Suppression of ( f ) copGFP-Polβ(WT) or ( g ) copGFP-Polβ(TM) recruitment to DNA damage-induced foci by the PARP inhibitors ABT-888, PJ34 and BMN-673. Stable LN428 cells expressing copGFP-Polβ(WT) or/and copGFP-Polβ(TM) were pre-treated with PARP inhibitors (PJ34, 4 μM; ABT-888, 10 μM; or BMN-673, 5 μM) for 1 h or without PARP inhibitor treatment, then cells were exposed to the 405-nm laser (50 ms or 1,000 ms). Images of cells were obtained after 2 min laser treatment. Results indicate mean±s.d. of five to eight independent cells. A one-tailed t -test was used for the statistical analysis and the P value was determined comparing cells treated with the PARP inhibitors as compared with cells without PARP inhibitor treatment. Full size image In the second approach, we visualized BER protein recruitment following exposure to 405 nm laser light, as was described previously for the analysis of BER protein recruitment [27] . Using this system, we also evaluated the role for XRCC1 in the recruitment of the WT and TM mutant of Polβ by depleting XRCC1 via lentiviral-mediated expression of short hairpin RNA (shRNA; Supplementary Fig. 7A ). Previous reports suggested that the recruitment of Polβ to DNA damage sites is XRCC1 dependent [27] . In line with these earlier reports, we also find that the foci intensity of copGFP-Polβ(TM) is weaker than copGFP-Polβ(WT) following damage induction using the 405 nm laser light ( Fig. 2d,e ; Supplementary Fig. 2B ). To test whether the recruitment of Polβ is XRCC1 dependent while the recruitment of the mutant, Polβ(TM), is XRCC1 independent, stable LN428 cells expressing copGFP-Polβ(WT) or copGFP-Polβ(TM) (with or without XRCC1 expression; Supplementary Figs 2A and 7A ) were laser irradiated (405 nm) and foci intensity was quantified. Further, we find that the steady-state levels ( Fig. 3b ) and recruitment of copGFP-Polβ(WT) are significantly decreased when XRCC1 is depleted ( Fig. 2d,e ; Supplementary Fig. 2B ). Similar to the KillerRed approach ( Fig. 2c ), the foci intensity of the mutant, copGFP-Polβ(TM), is also reduced as compared with copGFP-Polβ(WT) and the loss of XRCC1 does not impact the recruitment of the Polβ mutant, copGFP-Polβ(TM) ( Fig. 2d,e ; Supplementary Fig. 2B ). 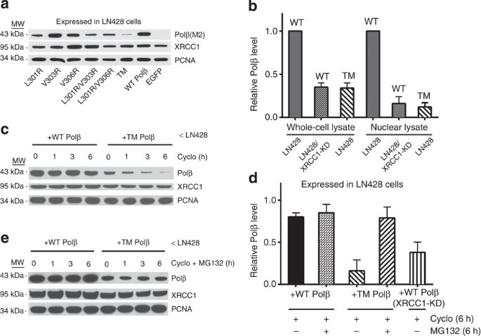Figure 3: DNA polymerase β stability depends on complex formation with XRCC1. (a) Immunoblot of nuclear lysates from stable LN428 cell lines expressing Flag-Polβ(WT) or the V303 loop mutants (as indicated), probing for the steady-state levels of Flag-Polβ, XRCC1 and PCNA, as indicated. A representative immunoblot image is shown. (b) The relative level of Flag-Polβ in WCLs and nuclear lysates from stable LN428 cell lines expressing Flag-Polβ(WT) or Flag-Polβ(TM) and from stable LN428/XRCC1-KD cells expressing Flag-Polβ(WT), as determined by immunoblot analysis, as inaandSupplementary Fig. 3D. The result indicates mean±s.d. of two independent experiments. (c) Immunoblot of WCLs from stable LN428 cell lines expressing Flag-Polβ(WT) or Flag-Polβ(TM) after exposure to cycloheximide (Cyclo) for the times indicated. The immunoblot image depicts the levels of Flag-Polβ, XRCC1 and PCNA, before and after treatment with Cyclo, showing the stability of Flag-Polβ(WT) and the rapid degradation of Flag-Polβ(TM). A representative immunoblot image is shown. (d) The relative level of Flag-Polβ in WCLs from stable LN428 cell lines expressing Flag-Polβ(WT) or Flag-Polβ(TM) and from stable LN428/XRCC1-KD cells expressing Flag-Polβ(WT). Cells were treated with Cyclo or Cyclo+MG132 (6 h) and protein levels determined by immunoblot analysis, as ine. The result indicates mean±s.d. of two independent experiments. (e) Immunoblot of WCLs from stable LN428 cell lines expressing Flag-Polβ(WT) or Flag-Polβ(TM) after exposure to Cyclo+the proteasome inhibitor MG132 for the times indicated. The immunoblot image depicts the levels of Flag-Polβ, XRCC1 and PCNA, before and after treatment with Cyclo+MG132, showing the stability of Flag-Polβ(WT) and the restored stability of Flag-Polβ(TM) due to proteasome inhibition. A representative immunoblot image is shown. See alsoSupplementary Figs 8, 9. Figure 3: DNA polymerase β stability depends on complex formation with XRCC1. ( a ) Immunoblot of nuclear lysates from stable LN428 cell lines expressing Flag-Polβ(WT) or the V303 loop mutants (as indicated), probing for the steady-state levels of Flag-Polβ, XRCC1 and PCNA, as indicated. A representative immunoblot image is shown. ( b ) The relative level of Flag-Polβ in WCLs and nuclear lysates from stable LN428 cell lines expressing Flag-Polβ(WT) or Flag-Polβ(TM) and from stable LN428/XRCC1-KD cells expressing Flag-Polβ(WT), as determined by immunoblot analysis, as in a and Supplementary Fig. 3D . The result indicates mean±s.d. of two independent experiments. ( c ) Immunoblot of WCLs from stable LN428 cell lines expressing Flag-Polβ(WT) or Flag-Polβ(TM) after exposure to cycloheximide (Cyclo) for the times indicated. The immunoblot image depicts the levels of Flag-Polβ, XRCC1 and PCNA, before and after treatment with Cyclo, showing the stability of Flag-Polβ(WT) and the rapid degradation of Flag-Polβ(TM). A representative immunoblot image is shown. ( d ) The relative level of Flag-Polβ in WCLs from stable LN428 cell lines expressing Flag-Polβ(WT) or Flag-Polβ(TM) and from stable LN428/XRCC1-KD cells expressing Flag-Polβ(WT). Cells were treated with Cyclo or Cyclo+MG132 (6 h) and protein levels determined by immunoblot analysis, as in e . The result indicates mean±s.d. of two independent experiments. ( e ) Immunoblot of WCLs from stable LN428 cell lines expressing Flag-Polβ(WT) or Flag-Polβ(TM) after exposure to Cyclo+the proteasome inhibitor MG132 for the times indicated. The immunoblot image depicts the levels of Flag-Polβ, XRCC1 and PCNA, before and after treatment with Cyclo+MG132, showing the stability of Flag-Polβ(WT) and the restored stability of Flag-Polβ(TM) due to proteasome inhibition. A representative immunoblot image is shown. See also Supplementary Figs 8, 9 . Full size image Given the important role for XRCC1 in recruiting Polβ to sites of damage and the requirement for PARP1 to facilitate recruitment of XRCC1, we next evaluated a role for PARP1 activation. Whereas close to 50% of the KillerRed-induced foci intensity from copGFP-Polβ(WT) is lost on PARP inhibition, only a small fraction of the foci intensity from copGFP-Polβ(TM) is affected ( Fig. 2c ). Similarly, the laser-induced recruitment of copGFP-Polβ(WT) is significantly reduced when the cells are pre-treated with ABT-888 or BMN-673 ( Fig. 2f ), both clinically useful PARP inhibitors [28] . Interestingly, laser-induced recruitment of copGFP-Polβ(TM) is also affected by PARP inhibition ( Fig. 2g ). Taken together, these data suggest that the disruption of the Polβ/XRCC1 interaction allows the recruitment of cellular BER proteins to form DNA repair foci, albeit at a lower level. This supports our results ( Fig. 1 ) and hypothesis that this interaction is not essential for the cellular response to DNA damage. Polβ stability depends on complex formation with XRCC1 We observed that the steady-state levels of the Polβ V303 loop mutant proteins were decreased as compared with that of Flag-Polβ(WT). Importantly, protein levels of the mutants were inversely proportional to the ability of each to form a Polβ/XRCC1 complex ( Fig. 3a ; Supplementary Fig. 3A,B ). In contrast, analysis by quantitative reverse transcription PCR (qRT–PCR) showed no difference in the mRNA expression levels between Flag-Polβ(WT) and the V303 loop mutant Flag-Polβ(TM) ( Supplementary Fig. 3C ). We therefore tested the hypothesis that the stability of Polβ protein depends on the Polβ/XRCC1 interaction and is the result of proteasome-mediated degradation. In line with this hypothesis, we found that Flag-Polβ(WT) is unstable when XRCC1 levels are reduced by RNA interference ( Fig. 3b ; Supplementary Fig. 3D ). When comparing cells expressing Flag-Polβ(WT) to those expressing Flag-Polβ(TM) in the presence of the protein synthesis inhibitor cycloheximide, the level of Flag-Polβ(WT) protein remained essentially constant, reflecting the stability of the WT form of Polβ ( Fig. 3c,d ). However, the expression level of the XRCC1 interaction mutant, Flag-Polβ(TM), was reduced by 50% after 1 h exposure to cycloheximide and >90% reduced at 6 h ( Fig. 3c,d ). We conclude that the instability of Flag-Polβ(TM) is the result of proteasome-mediated degradation since treatment with the proteasome-inhibitor MG132 stabilizes Flag-Polβ(TM) protein levels ( Fig. 3d,e ). Together, these data suggest that the interaction with XRCC1 promotes Polβ stability by preventing proteasome-mediated degradation. Protein degradation via the proteasome is often mediated by poly-ubiquitylation [29] . We next determined whether Polβ, when not bound to XRCC1, is ubiquitylated. By co-expression of HA-ubiquitin in cells expressing Flag-Polβ(TM), we observed that Flag-Polβ(TM) is poly-ubiquitylated, suggesting that this promotes the degradation of Polβ ( Fig. 4a ). Polβ mono-ubiquitylation by MULE on residues K41, K61 and K81 followed by CHIP-mediated poly-ubiquitylation on the N terminus was recently reported [30] , [31] . Therefore, we investigated the role of MULE and CHIP in the ubiquitylation of Polβ when not bound to XRCC1. Mutation of the reported MULE target residues K41, K61 and K81 (K41R/K61R/K81R; referred to herein as KTM) in WT Flag-Polβ does not impact stability ( Supplementary Fig. 3E , top panel). Altering these MULE target residues in Flag-Polβ(TM) (Flag-Polβ(TM/KTM)) does not rescue the proteasome-mediated instability resulting from an inability to interact with XRCC1 ( Supplementary Fig. 3E , middle, bottom panels). The data presented here would imply that Polβ is not targeted for degradation by modification of the N-terminal residues K41, K61 and K81, suggesting that Polβ may be targeted for degradation at alternate sites. We observed that the C-terminal domain of Polβ (residues 91–335), when expressed in XRCC1-KD cells, is rapidly degraded, suggesting that the site of ubiquitylation is in the C terminus ( Supplementary Fig. 3F ). 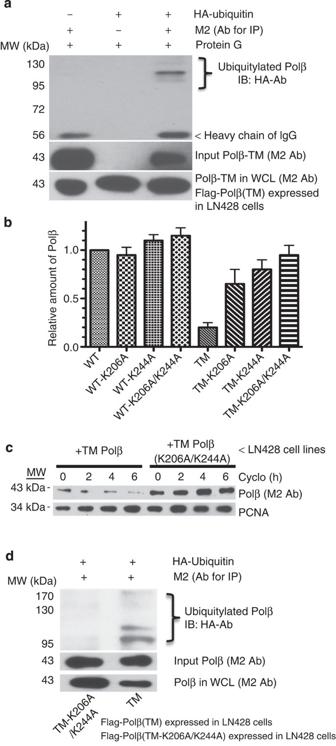Figure 4: The C-terminal domain of DNA polymerase β is targeted for proteasome-mediated degradation by ubiquitylation on K206/K244. (a) Immunoblot of WCLs from stable LN428 cell lines expressing Flag-Polβ(TM) after expression of HA-ubiquitin. Flag-Polβ(TM) was isolated by IP and probed for the HA-ubiquitin modification by immunoblot with the HA-Ab. The level of Flag-Polβ(TM) in the WCL and the input level of Flag-Polβ(TM) is detected using the M2 Flag-Ab. (b) The relative level of Flag-Polβ in WCLs from stable LN428 cell lines expressing Flag-Polβ(WT), Flag-Polβ(TM) and the indicated K206A, K244A or K206A/K244A mutants. The predicted ubiquitylation sites K206 and K244 reverse the instability of Flag-Polβ(TM), as determined by immunoblot analysis, as inSupplementary Fig. 4D. The result indicates mean±s.d. of two independent experiments. (c) Immunoblot of WCLs from stable LN428 cell lines expressing Flag-Polβ(TM) or Flag-Polβ(TM/K206A/K244A) after exposure to Cyclo for the times indicated. The immunoblot image depicts the levels of Flag-Polβ, XRCC1 and PCNA, before and after treatment with Cyclo, showing the rapid degradation of Flag-Polβ(TM) and the stability of Flag-Polβ(TM/K206A/K244A). A representative immunoblot image is shown. For quantified results, seeSupplementary Fig. 4E. (d) Immunoblot of WCLs from stable LN428 cell lines expressing Flag-Polβ(TM) or Flag-Polβ(TM/K206A/K244A) after expression of HA-ubiquitin. Flag-Polβ(TM) or Flag-Polβ(TM/K206A/K244A) was isolated by IP and probed for the HA-ubiquitin modification by immunoblot with the HA-Ab, showing the ubiquitylation of Flag-Polβ(TM) but not Flag-Polβ(TM/K206A/K244A). The level of Flag-Polβ(TM) or Flag-Polβ(TM/K206A/K244A) in the WCLs and the input level of Flag-Polβ(TM) or Flag-Polβ(TM/K206A/K244A) are detected using the M2 Flag-Ab. Figure 4: The C-terminal domain of DNA polymerase β is targeted for proteasome-mediated degradation by ubiquitylation on K206/K244. ( a ) Immunoblot of WCLs from stable LN428 cell lines expressing Flag-Polβ(TM) after expression of HA-ubiquitin. Flag-Polβ(TM) was isolated by IP and probed for the HA-ubiquitin modification by immunoblot with the HA-Ab. The level of Flag-Polβ(TM) in the WCL and the input level of Flag-Polβ(TM) is detected using the M2 Flag-Ab. ( b ) The relative level of Flag-Polβ in WCLs from stable LN428 cell lines expressing Flag-Polβ(WT), Flag-Polβ(TM) and the indicated K206A, K244A or K206A/K244A mutants. The predicted ubiquitylation sites K206 and K244 reverse the instability of Flag-Polβ(TM), as determined by immunoblot analysis, as in Supplementary Fig. 4D . The result indicates mean±s.d. of two independent experiments. ( c ) Immunoblot of WCLs from stable LN428 cell lines expressing Flag-Polβ(TM) or Flag-Polβ(TM/K206A/K244A) after exposure to Cyclo for the times indicated. The immunoblot image depicts the levels of Flag-Polβ, XRCC1 and PCNA, before and after treatment with Cyclo, showing the rapid degradation of Flag-Polβ(TM) and the stability of Flag-Polβ(TM/K206A/K244A). A representative immunoblot image is shown. For quantified results, see Supplementary Fig. 4E . ( d ) Immunoblot of WCLs from stable LN428 cell lines expressing Flag-Polβ(TM) or Flag-Polβ(TM/K206A/K244A) after expression of HA-ubiquitin. Flag-Polβ(TM) or Flag-Polβ(TM/K206A/K244A) was isolated by IP and probed for the HA-ubiquitin modification by immunoblot with the HA-Ab, showing the ubiquitylation of Flag-Polβ(TM) but not Flag-Polβ(TM/K206A/K244A). The level of Flag-Polβ(TM) or Flag-Polβ(TM/K206A/K244A) in the WCLs and the input level of Flag-Polβ(TM) or Flag-Polβ(TM/K206A/K244A) are detected using the M2 Flag-Ab. Full size image In earlier studies, Polβ was suggested to be a target of the E3 ligase CHIP [30] , [31] . We therefore next modulated the expression of CHIP, via overexpression and shRNA-mediated knockdown, to determine whether the degradation of Polβ is mediated by CHIP. Overexpression of Flag-CHIP had no effect on the stability of Flag-Polβ(WT) ( Supplementary Fig. 4A ) and did not enhance the degradation of Flag-Polβ(TM) ( Supplementary Fig. 4A,B ). Finally, we depleted LN428/Flag-Polβ(TM) cells of CHIP using two different CHIP-shRNAs ( Supplementary Fig. 4C ). Following loss of CHIP protein, we were unable to observe a change in the instability of the V303 loop mutant of Polβ, Flag-Polβ(TM), even in the presence of cycloheximide ( Supplementary Fig. 4C ). In summary, these findings suggest that Polβ is ubiquitylated on the C terminus and proteasome-mediated degradation of Polβ, when not bound to XRCC1, is independent of CHIP. The observation that Polβ is likely ubiquitylated on the C terminus (see Supplementary Fig. 3F ) prompted us to evaluate potential ubiquitylation sites for the complete Polβ amino-acid sequence. Analysis utilizing the UbPred software tool ( http://www.ubpred.org ) [32] predicted two potential ubiquitylation sites, each localized to the C-terminal domain of Polβ: K206 and K244. To determine whether the K206 and/or K244 residues were indeed ubiquitylated to promote Polβ degradation when not bound to XRCC1, we compared WT and TM Polβ protein levels in cell lines expressing mutant Polβ proteins: Flag-Polβ(K206A), Flag-Polβ(K244A), Flag-Polβ(K206A/K244A), Flag-Polβ(TM/K206A), Flag-Polβ(TM/K244A) and Flag-Polβ(TM/K206A/K244A). Confirming a role for these residues (K206A and K244A) in the stability of Flag-Polβ(TM) ( Supplementary Fig. 4D ), we observed a marked increase in basal protein levels when the Flag-Polβ(TM) was mutated at both sites (K206A/K244A), restoring the level of Flag-Polβ(TM) protein to a level similar to Flag-Polβ(WT) ( Fig. 4b ). Comparison of cells expressing Flag-Polβ(TM/K206A/K244A) to those expressing Flag-Polβ(TM), in the presence of cycloheximide, further emphasizes the stability that is imposed by mutating residues K206 and K244 ( Fig. 4c ; Supplementary Fig. 4E ). We conclude from these studies that amino-acid residues K206 and K244 are the ubiquitylation sites observed in the Flag-Polβ(TM) protein that are modified due to an inability to bind to XRCC1 ( Fig. 4d ). When the Flag-Polβ(TM) protein is mutated at K206/K244, expression levels return to normal and the Flag-Polβ(TM/K206A/K244A) protein is still unable to bind to XRCC1 ( Supplementary Fig. 4F ). Overall, these studies demonstrate that Polβ stability in human cells depends on binding to XRCC1 and once separated from XRCC1, Polβ is ubiquitylated on K206 and K244 and targeted for proteasome-mediated degradation. Unbound XRCC1 is an HSP90 client protein Earlier biochemical analysis of proteins involved in BER implicated heat–shock chaperone proteins, but their role was never elucidated [33] , [34] , [35] , [36] , [37] . Further, it has been suggested that HSP90 may interact with DNA repair and related DNA metabolic proteins via co-chaperones [38] or on phosphorylation [39] . In many cases, heat–shock chaperone (HSP90) client proteins are protected from ubiquitylation [40] . We questioned whether the chaperone HSP90 is bound to and thereby protecting either Flag-Polβ(WT) or Flag-Polβ(TM) from CHIP-mediated ubiquitylation in vivo . To test the hypothesis that Polβ might be an HSP90 client protein, we expressed HA-HSP90 in cells expressing Flag-Polβ(WT) or Flag-Polβ(TM) and analysed BER proteins bound to HSP90 ( Supplementary Fig. 5C ). However, we did not find Polβ (neither the WT form nor the mutant, TM) in a complex with HSP90, ruling out a possible role of HSP90 in the protection of CHIP-mediated degradation of Polβ. Surprisingly, we find that XRCC1 is bound to HA-HSP90 but only in cells either deficient in Polβ or expressing the XRCC1 interaction-deficient mutant, Flag-Polβ(TM) ( Supplementary Fig. 5C ). We observed this in both of the human tumour cell lines LN428 and T98G. To determine whether endogenous HSP90 interacts with XRCC1 and other BER-related proteins, we immunoprecipitated HSP90 from lysates of cells with a Polβ-deficient background (T98G/MPG/PolβKD), expressing EGFP, Polβ(WT) or Polβ(TM), and examined BER proteins bound to endogenous HSP90. We confirmed that XRCC1 binds to endogenously expressed HSP90 in cells expressing either EGFP or Polβ(TM) but not in those cells expressing Polβ(WT) ( Fig. 5a ). However, the interaction between HSP90 and XRCC1 was unique among BER proteins. Neither PARP1, MPG and APE1 nor PCNA were found to bind to HSP90 ( Fig. 5a ), suggesting that the XRCC1/HSP90 complex is selective and may play a role in XRCC1-dependent and Polβ-independent DNA repair. To confirm the Polβ-dependent complex formation between XRCC1 and HSP90 in cells with endogenous levels of Polβ, we analysed mouse embryonic fibroblasts (MEFs) proficient or deficient for Polβ [41] . Importantly, we observed a robust interaction between XRCC1 and HSP90 in Polβ KO (88TAg) MEFs that was abolished in the Polβ-proficient isogenic WT MEFs (92TAg) ( Fig. 5b ; Supplementary Fig. 5A ). Interestingly, when purified recombinant Polβ was added to the Polβ KO lysates, the XRCC1/HSP90 complex is lost and we see a re-assembly of the Polβ/XRCC1 complex ( Supplementary Fig. 5B ), suggesting that HPS90 may also function to assemble the Polβ/XRCC1 complex. Overall, these data indicate that free XRCC1 (not bound to Polβ) and HSP90 form a heterodimeric complex (XRCC1/HSP90) in multiple mammalian species. 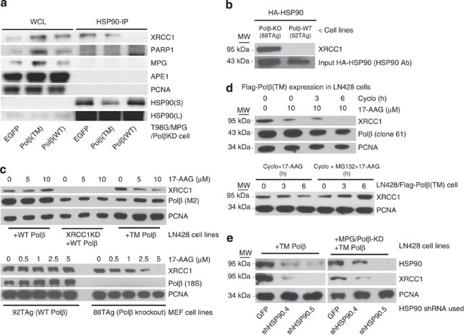Figure 5: Unbound XRCC1 is an HSP90 client protein. (a) HSP90 interacts with XRCC1 but not other BER-related proteins. WCL were prepared from proliferating T98G/MPG/Polβ-KD cells expressing EGFP, Flag-Polβ(WT) or Flag-Polβ(TM) (left panel). XRCC1 and other BER-related proteins were immunoprecipitated with an HSP90 antibody and examined by immunoblot as shown (right panel). (b) HA-HSP90 interacts with XRCC1 in Polβ-KO MEFs, not in WT MEFs. WT (92TAg) and Polβ-KO (88TAg) MEFs, after expression of HA-HSP90, were probed for HSP90-interacting proteins by IP of the expressed HA-HSP90 via the N-terminal HA epitope tag and probing for XRCC1 by immunoblot. Input HA-HSP90 is also shown. (c) HSP90 inhibitor 17-AAG treatment induces the degradation of XRCC1 in cells lacking Polβ (LN428/Polβ-KD cells and MEFs), as indicated: immunoblot of WCLs from stable LN428 cell lines expressing Flag-Polβ(WT) or Flag-Polβ(TM) and from stable LN428/XRCC1-KD cells expressing Flag-Polβ(WT) (shown in top panel) and immunoblot of WCLs from WT (92TAg) and Polβ-KO (88TAg) MEFs (shown in bottom panel) after exposure to 17-AAG at the concentrations indicated. The immunoblot image depicts the levels of XRCC1, Flag-Polβ and PCNA, before and after treatment with 17-AAG. A representative immunoblot image is shown. For quantified results, seeSupplementary Fig. 5D,E. (d) Cycloheximide-enhanced degradation of XRCC1 in LN428/Flag-Polβ(TM) cells treated with 17-AAG is protected by MG132: (top panel) immunoblot of WCLs from stable LN428 cell lines expressing Flag-Polβ(TM) after exposure to 17-AAG (0 or 10 μM, as indicated) and cycloheximide (Cyclo) for the times indicated. A representative immunoblot image is shown. (Bottom panel) Immunoblot of WCLs from stable T98G/Polβ-KD cell lines expressing EGFP after exposure to 17-AAG (10 μM) and Cyclo or Cyclo+MG132 for the times indicated. A representative image is shown. For quantified results, seeSupplementary Fig. 5F. (e) HSP90 knockdown induces the degradation of XRCC1 in LN428/Flag-Polβ(TM) and LN428/MPG/Polβ-KD/Flag-Polβ(TM) cells: immunoblot of WCLs from LN428 cell lines expressing Flag-Polβ(TM) or LN428/MPG/Polβ-KD cells expressing Flag-Polβ(TM) after lentiviral-mediated expression of GFP or HSP90-specific shRNA, as indicated. A representative immunoblot image is shown. Figure 5: Unbound XRCC1 is an HSP90 client protein. ( a ) HSP90 interacts with XRCC1 but not other BER-related proteins. WCL were prepared from proliferating T98G/MPG/Polβ-KD cells expressing EGFP, Flag-Polβ(WT) or Flag-Polβ(TM) (left panel). XRCC1 and other BER-related proteins were immunoprecipitated with an HSP90 antibody and examined by immunoblot as shown (right panel). ( b ) HA-HSP90 interacts with XRCC1 in Polβ-KO MEFs, not in WT MEFs. WT (92TAg) and Polβ-KO (88TAg) MEFs, after expression of HA-HSP90, were probed for HSP90-interacting proteins by IP of the expressed HA-HSP90 via the N-terminal HA epitope tag and probing for XRCC1 by immunoblot. Input HA-HSP90 is also shown. ( c ) HSP90 inhibitor 17-AAG treatment induces the degradation of XRCC1 in cells lacking Polβ (LN428/Polβ-KD cells and MEFs), as indicated: immunoblot of WCLs from stable LN428 cell lines expressing Flag-Polβ(WT) or Flag-Polβ(TM) and from stable LN428/XRCC1-KD cells expressing Flag-Polβ(WT) (shown in top panel) and immunoblot of WCLs from WT (92TAg) and Polβ-KO (88TAg) MEFs (shown in bottom panel) after exposure to 17-AAG at the concentrations indicated. The immunoblot image depicts the levels of XRCC1, Flag-Polβ and PCNA, before and after treatment with 17-AAG. A representative immunoblot image is shown. For quantified results, see Supplementary Fig. 5D,E . ( d ) Cycloheximide-enhanced degradation of XRCC1 in LN428/Flag-Polβ(TM) cells treated with 17-AAG is protected by MG132: (top panel) immunoblot of WCLs from stable LN428 cell lines expressing Flag-Polβ(TM) after exposure to 17-AAG (0 or 10 μM, as indicated) and cycloheximide (Cyclo) for the times indicated. A representative immunoblot image is shown. (Bottom panel) Immunoblot of WCLs from stable T98G/Polβ-KD cell lines expressing EGFP after exposure to 17-AAG (10 μM) and Cyclo or Cyclo+MG132 for the times indicated. A representative image is shown. For quantified results, see Supplementary Fig. 5F . ( e ) HSP90 knockdown induces the degradation of XRCC1 in LN428/Flag-Polβ(TM) and LN428/MPG/Polβ-KD/Flag-Polβ(TM) cells: immunoblot of WCLs from LN428 cell lines expressing Flag-Polβ(TM) or LN428/MPG/Polβ-KD cells expressing Flag-Polβ(TM) after lentiviral-mediated expression of GFP or HSP90-specific shRNA, as indicated. A representative immunoblot image is shown. Full size image The discovery that free XRCC1 (not bound to Polβ) is an HSP90 client protein therefore implicates HSP90 as a regulator of XRCC1, protecting XRCC1 from proteasome-mediated degradation. On HSP90 inhibition, free XRCC1 would be expected to be an unstable protein. To test this hypothesis, we treated cells with the HSP90 inhibitor 17-allylamino-17-demethoxygeldanamycin (17-AAG; Fig. 5c , top). Treatment with increasing concentrations of 17-AAG had no effect on the stability of XRCC1 in cells expressing Flag-Polβ(WT). However, consistent with a role for HSP90, 17-AAG treatment resulted in a dose-dependent decrease in XRCC1 protein levels in cells expressing the XRCC1 interaction-deficient mutant Flag-Polβ(TM) ( Fig. 5c , top; Supplementary Fig. 5D ). Similarly, treatment of MEFs that express endogenous Polβ (92TAg) with 17-AAG had no affect on XRCC1 protein stability, yet 17-AAG treatment of the Polβ-KO MEFs (88TAg) led to complete loss of XRCC1 ( Fig. 5c , bottom; Supplementary Fig. 5E ). This 17-AAG-induced loss of XRCC1 protein levels, in LN428 cells expressing Flag-Polβ(TM), is enhanced in the presence of cycloheximide ( Fig. 5d , top; Supplementary Fig. 5F ) and is reversed when MG132 is added ( Fig. 5d , bottom). In addition to HSP90 inhibition, we further show that depletion of HSP90 also triggers XRCC1 protein loss in the Flag-Polβ(TM)-expressing LN428 cells ( Fig. 5e ). In all, we have shown that Polβ and XRCC1 form a strong heterodimeric complex that contributes to protein stability of both proteins. Disruption of the Polβ/XRCC1 interaction promotes proteasome-mediated degradation of Polβ and the formation of a second heterodimer comprised of XRCC1 and HSP90. These studies implicate a novel role for HSP90 in protecting free XRCC1 from ubiquitylation and proteasome-mediated degradation when not bound to Polβ and suggest that XRCC1 may exist in multiple heterodimer complexes. CHIP-mediated degradation of XRCC1 is regulated by HSP90 These data suggest that the ubiquitin-proteasome pathway is involved in the degradation of XRCC1 (when not bound to the chaperone HSP90 or Polβ). CHIP is a major E3 ubiquitin ligase that targets and mediates the degradation of HSP90 client proteins [42] ; thus, most are further degraded following overexpression of CHIP [43] . We first determined whether CHIP overexpression enhanced the degradation of XRCC1 when exposed to 17-AAG. Whereas overexpression of CHIP had little to no effect on the steady-state levels of XRCC1, these levels were reduced (by half) in all cells when also exposed to 17-AAG ( Fig. 6a,b ). In addition, knockdown of CHIP suppresses the 17-AAG-mediated loss of XRCC1 ( Fig. 6c ). Consistent with the data presented above ( Fig. 5 ), 17-AAG promoted the degradation of XRCC1 in a manner dependent on its ability to interact with Polβ. However, CHIP overexpression did not enhance the degradation of XRCC1 in a Polβ-binding-dependent manner. These data suggest that an additional 17-AAG-dependent process is responsible for the proteasome-mediated degradation of the pool of XRCC1 not bound to Polβ. Overall, these results not only clearly support a role for CHIP in the degradation of XRCC1 and establish that CHIP-mediated degradation of XRCC1 is regulated by the activity and availability of HSP90, but also points to an as yet undetermined CHIP-independent mechanism of XRCC1 degradation. 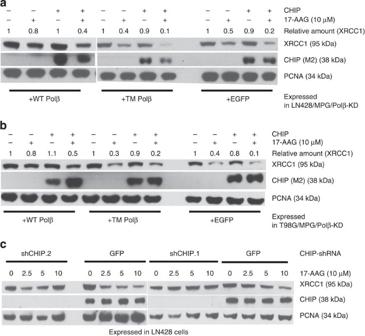Figure 6: CHIP-mediated degradation of XRCC1 is regulated by HSP90. Overexpression of the E3 ligase CHIP enhances the 17-AAG-mediated degradation of XRCC1 in (a) LN428/MPG/Polβ-KD/Flag-Polβ(TM) cells and (b) T98G/MPG/Polβ-KD/Flag-Polβ(TM) cells: immunoblot of WCLs from stable LN428/MPG/Polβ-KD cell lines (a) or T98G/MPG/Polβ-KD/Flag-Polβ(TM) cell lines (b) expressing Flag-Polβ(WT), Flag-Polβ(TM) or EGFP after exposure to 17-AAG at the concentrations indicated and after overexpression of CHIP, as indicated. The immunoblot images depict the levels of XRCC1, CHIP and PCNA, before and after treatment with 17-AAG, showing the stability of XRCC1 in the cells expressing Flag-Polβ(WT) and the rapid degradation of XRCC1 in the cells expressing Flag-Polβ(TM) or EGFP. Representative immunoblot images are shown. (c) CHIP knockdown efficiently prevents 17-AAG-mediated degradation of XRCC1 in LN428 cells: immunoblot of WCLs from stable LN428 cells expressing CHIP-specific shRNA (shCHIP.2 or shCHIP.1) or GFP (control) after exposure to 17-AAG at the concentration indicated. The immunoblot image shows the level of XRCC1, CHIP and PCNA (loading control), before and after treatment with 17-AAG. Figure 6: CHIP-mediated degradation of XRCC1 is regulated by HSP90. Overexpression of the E3 ligase CHIP enhances the 17-AAG-mediated degradation of XRCC1 in ( a ) LN428/MPG/Polβ-KD/Flag-Polβ(TM) cells and ( b ) T98G/MPG/Polβ-KD/Flag-Polβ(TM) cells: immunoblot of WCLs from stable LN428/MPG/Polβ-KD cell lines ( a ) or T98G/MPG/Polβ-KD/Flag-Polβ(TM) cell lines ( b ) expressing Flag-Polβ(WT), Flag-Polβ(TM) or EGFP after exposure to 17-AAG at the concentrations indicated and after overexpression of CHIP, as indicated. The immunoblot images depict the levels of XRCC1, CHIP and PCNA, before and after treatment with 17-AAG, showing the stability of XRCC1 in the cells expressing Flag-Polβ(WT) and the rapid degradation of XRCC1 in the cells expressing Flag-Polβ(TM) or EGFP. Representative immunoblot images are shown. ( c ) CHIP knockdown efficiently prevents 17-AAG-mediated degradation of XRCC1 in LN428 cells: immunoblot of WCLs from stable LN428 cells expressing CHIP-specific shRNA (shCHIP.2 or shCHIP.1) or GFP (control) after exposure to 17-AAG at the concentration indicated. The immunoblot image shows the level of XRCC1, CHIP and PCNA (loading control), before and after treatment with 17-AAG. Full size image DNA damage and cell cycle regulate the XRCC1/HSP90 complex XRCC1 and Polβ have potentially unique roles in DNA repair and development. Our observation that XRCC1 is protected from degradation by complexing with HSP90 in a Polβ-binding-dependent manner prompted us to further evaluate the role of this complex in essential cellular processes. Indeed, cellular survival, in response to different DNA-damaging agents, reveals distinct roles for Polβ and XRCC1 that supports an XRCC1 function that is different from Polβ and hence, potentially independent of Polβ binding. As shown in Fig. 7a , loss of Polβ has a greater impact than the loss of XRCC1 (~80% knockdown, shown in Supplementary Fig. 7A ) on cellular survival in response to MNNG, while the involvement or requirement for Polβ and XRCC1 is similar in response to H 2 O 2 and IR. Supporting our suggestion that Polβ and XRCC1 may have separate functions depending on the type of DNA damage, we show that the combined loss of Polβ and XRCC1 has a stronger sensitization effect in response to H 2 O 2 than in response to MNNG. However, in line with earlier reports [44] , [45] , the loss of XRCC1 sensitizes these cells significantly to these agents in cells expressing either Flag-Polβ(WT) or Flag-Polβ(TM). These observations therefore prompted us to assess Polβ/XRCC1 and XRCC1/HSP90 complex formation following treatment with different damaging agents. In addition, prior reports demonstrated that the requirement for Polβ may depend on the cell cycle. In response to IR, mouse fibroblasts respond differently when proliferating or confluent [46] , [47] . In contrast to cells deficient in XRCC1, the requirement for Polβ in repair and survival is confined to confluent or G1 cells, suggesting alternative XRCC1-mediated repair in S-phase. This prompted us to test whether the Polβ/XRCC1 complex is primarily required in confluent cells at the cost of the XRCC1/HSP90 complex that may enable Polβ-independent repair in proliferating cells and whether this is altered in response to DNA damage. Consistent with this hypothesis, the occurrence of the Polβ/XRCC1 complex is greater in confluent cells, whereas the XRCC1/HSP90 complex is primarily evident in proliferating cells ( Fig. 7b ; Supplementary Figs 5A and 6A ). 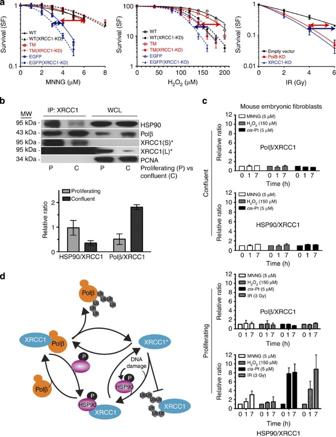Figure 7: Dynamic interaction of DNA polymerase β and HSP90 with XRCC1 regulates BER sub-pathway choice. (a) Cell viability in response to MNNG, H2O2or IR. Left panel: LN428/MPG or LN428/MPG/XRCC1-KD cells expressing Flag-Polβ(WT), Flag-Polβ(TM) or EGFP after MNNG treatment, as measured by the MTS assay 48 h after exposure. Results indicate the mean±s.d. of three independent experiments. Middle panel: LN428 or LN428/XRCC1-KD cells expressing Flag-Polβ(WT), Flag-Polβ(TM) or EGFP after H2O2treatment, as measured by the CyQuant assay 10 days after exposure. Results indicate the mean±s.d. of three independent experiments. Right panel: Clonogenic survival assay of LN428/Polβ-KD, LN428/Puro and LN428/XRCC1-KD cells after exposure to IR. Data points represent means and s.d. of at least three experiments, each performed in triplicate. The arrows indicate the extent of the requirement for Polβ (red) or XRCC1 (blue). Plots show the relative surviving fraction as compared with untreated cells. (b) Polβ/XRCC1 and XRCC1/HSP90 heterodimer ratios in proliferating (P) and confluent (C) MEFs (92TAg) were probed for heterodimer formation by IP of XRCC1 (XRCC1-Ab) and probing for XRCC1, HSP90 and Polβ by immunoblot. A representative immunoblot is shown. *¼ input IP product for XRCC1; L, longer exposure time; S, short exposure time. Bar graphs are plotted with mean±s.d. of two independent experiments. (c) The relative ratio of Polβ/XRCC1 and HSP90/XRCC1 was quantified following IP of XRCC1 and analysis for Polβ or HSP90 (Supplementary Fig. 7C,E) from proliferating and confluent cells (92TAg MEFs) treated with different DNA-damaging agents. Bar graphs are plotted with mean±s.d. of two independent experiments. (d) Proposed model for the dynamic regulation of the stability and degradation of Polβ and XRCC1. Varied cellular conditions, such as HSP90 phosphorylation, alterations in the expression or function related to the cell cycle or DNA damage response and cell-type specificity promote the formation of one of the two heterodimers. Conditions that increase Polβ/XRCC1 levels would favour Polβ-dependent BER, whereas conditions that increase XRCC1/HSP90 levels would result in a preference for XRCC1-dependent or Polβ-independent BER. The degradation of XRCC1 is regulated by HSP90 and CHIP. Figure 7: Dynamic interaction of DNA polymerase β and HSP90 with XRCC1 regulates BER sub-pathway choice. ( a ) Cell viability in response to MNNG, H 2 O 2 or IR. Left panel: LN428/MPG or LN428/MPG/XRCC1-KD cells expressing Flag-Polβ(WT), Flag-Polβ(TM) or EGFP after MNNG treatment, as measured by the MTS assay 48 h after exposure. Results indicate the mean±s.d. of three independent experiments. Middle panel: LN428 or LN428/XRCC1-KD cells expressing Flag-Polβ(WT), Flag-Polβ(TM) or EGFP after H 2 O 2 treatment, as measured by the CyQuant assay 10 days after exposure. Results indicate the mean±s.d. of three independent experiments. Right panel: Clonogenic survival assay of LN428/Polβ-KD, LN428/Puro and LN428/XRCC1-KD cells after exposure to IR. Data points represent means and s.d. of at least three experiments, each performed in triplicate. The arrows indicate the extent of the requirement for Polβ (red) or XRCC1 (blue). Plots show the relative surviving fraction as compared with untreated cells. ( b ) Polβ/XRCC1 and XRCC1/HSP90 heterodimer ratios in proliferating (P) and confluent (C) MEFs (92TAg) were probed for heterodimer formation by IP of XRCC1 (XRCC1-Ab) and probing for XRCC1, HSP90 and Polβ by immunoblot. A representative immunoblot is shown. *¼ input IP product for XRCC1; L, longer exposure time; S, short exposure time. Bar graphs are plotted with mean±s.d. of two independent experiments. ( c ) The relative ratio of Polβ/XRCC1 and HSP90/XRCC1 was quantified following IP of XRCC1 and analysis for Polβ or HSP90 ( Supplementary Fig. 7C,E ) from proliferating and confluent cells (92TAg MEFs) treated with different DNA-damaging agents. Bar graphs are plotted with mean±s.d. of two independent experiments. ( d ) Proposed model for the dynamic regulation of the stability and degradation of Polβ and XRCC1. Varied cellular conditions, such as HSP90 phosphorylation, alterations in the expression or function related to the cell cycle or DNA damage response and cell-type specificity promote the formation of one of the two heterodimers. Conditions that increase Polβ/XRCC1 levels would favour Polβ-dependent BER, whereas conditions that increase XRCC1/HSP90 levels would result in a preference for XRCC1-dependent or Polβ-independent BER. The degradation of XRCC1 is regulated by HSP90 and CHIP. Full size image We found that HSP90 expression is quickly induced on DNA damage ( Supplementary Fig. 6B ). In response to varying DNA-damaging agents (MNNG, H 2 O 2 and cis -Pt), we observe a rapid induction of Polβ and a delayed induction of XRCC1. Consistent with its requirement for survival ( Fig. 7a ), the induction of Polβ in proliferating cells is only observed in response to MNNG and H 2 O 2 ( Supplementary Fig. 6B ). When evaluating the relative contribution of each heterodimer (Polβ/XRCC1 and XRCC1/HSP90), there is little impact on the overall status of the Polβ/XRCC1 complex ( Fig. 7c ; Supplementary Fig. 6C,E ). In contrast, there is a rapid increase in the appearance of the XRCC1/HSP90 complex on DNA damage. Interestingly, this is limited to proliferating cells and dependent on the type of damage (see Fig. 7c ; Supplementary Fig. 6B,C ). We did not observe a concomitant reduction of the Polβ/XRCC1 complex when the XRCC1/HSP90 complex is formed ( Fig. 7c ), as would be predicted by a hand-over mechanism. In fact, these data support the existence of a pool of XRCC1 in proliferating cells that is neither bound to Polβ nor HSP90 (denoted as XRCC1*, see Fig. 7d ). We note a different pattern of XRCC1/HSP90 complex formation in response to cis -Pt and IR ( Fig. 7c ; Supplementary Fig. 6C,E ). Assuming HSP90 functions to protect free XRCC1 from degradation, this observation points to the integration of XRCC1 in an alternate (active) repair complex on cis -Pt and IR exposure that does not include Polβ. Importantly, we find that the XRCC1/HSP90 complex has no apparent role in confluent cells ( Fig. 7b,c ; Supplementary Fig. 6E ). A functional role for HSP90, in XRCC1 stability and possibly XRCC1/Polβ ← XRCC1/HSP90 exchange, implicates a nuclear role for this factor. Although predominantly cytosolic, HSP90 has been implicated in nuclear retention of glucocorticoid receptor [48] . Most importantly, similar to XRCC1 (ref. 49 ), HSP90 is phosphorylated (on the N terminus; Thr5/7) by the DNA damage response kinase DNA-PK in response to DNA damage and accumulates in the nucleus [50] , [51] , [52] . We reasoned therefore that nuclear XRCC1 may complex with this phosphorylated isoform of HSP90, after DNA damage and/or during changes in the cell cycle. In line with our hypothesis, the level of pHSP90 is induced following treatment with either MNNG or cis -Pt in WT MEF cells (92TAg) ( Supplementary Fig. 7C ). Importantly, XRCC1 does complex with the pHSP90 isoform, phosphorylated on Thr5/7 ( Supplementary Fig. 7C ). A greater level of the pHSP90/XRCC1 dimer is formed in cells following treatment with cis -Pt than with MNNG ( Supplementary Fig. 7D ). This is consistent with the complex formation discussed above ( Fig. 7c ). In general, BER proteins are recruited within 30 min of DNA-damaging agent exposure [53] . However, the majority of DNA damage-induced induction of pHSP90 and XRCC1 and pHSP90/XRCC1 complex formation is observed after 1 h treatment ( Fig. 7c ; Supplementary Fig. 7C,D ). Further, we find that cis -Pt treatment results in more pHSP90/XRCC1 complex formation than following treatment with MNNG or H 2 O 2 ( Fig. 7c ; Supplementary Fig. 7B,C ) All together, these studies suggest that the (p)HSP90/XRCC1 complex may facilitate and promote a role for XRCC1 ( Fig. 7d ), together with other protein partners, in several DNA repair pathways independent of Polβ and BER. Indeed, we find, in Supplementary Fig. 5A , that complex formation between XRCC1 and HSP90 is both Polβ dependent and proliferation dependent. Specifically, as shown, Polβ governs XRCC1/HSP90 binding in proliferating cells only ( Supplementary Fig. 5A ), supporting a role for Polβ-independent repair in replication-associated repair processes. Overall, we suggest that the formation of the Polβ/XRCC1 and XRCC1/HSP90 heterodimers regulates DNA repair pathway choice and our studies support a novel functional component of BER that may facilitate this choice in response to DNA damage and cellular proliferation. Polβ and XRCC1 are essential BER proteins, with current models suggesting that they function as a static heterodimeric complex at sites of DNA repair. Tight binding between Polβ and XRCC1 provides the means for XRCC1-mediated recruitment of Polβ to foci of DNA damage and repair [3] , [4] , [54] . In contrast, XRCC1 and Polβ deficiency have drastically different phenotypes in mouse models, suggesting unique and independent functions for each. The Polβ-KO mouse survives gestation but is lethal just after birth [11] , whereas the XRCC1-KO mouse dies in an early stage of embryogenesis [12] . Whereas both proteins play a significant role together as a complex, mouse models suggest that Polβ and XRCC1 may have separate roles in mammalian development and cellular function. Understanding the regulation of this complex is critical to reveal the independent roles for each protein. BER models would predict that disrupting Polβ binding to XRCC1 impairs Polβ recruitment and function. Surprisingly, we find that Polβ is recruited to sites of DNA lesions from laser light, KillerRed ROS induction and MNNG ( Fig. 2 ; Supplementary Fig. 2B,C ) independent of its ability to bind to XRCC1. We do observe lower levels of recruitment for the mutant, Flag-Polβ(TM), as compared with the WT protein, but since the steady-state level of the mutant protein is suppressed (due to ubiquitylation and degradation; for example, Supplementary Fig. 3A,D ), it is formally possible that the decreased recruitment to sites of DNA damage may be a reflection of the decreased Polβ protein levels when mutated (TM) or when depleted of XRCC1. However, we find that the major phenotype associated with disruption of the Polβ/XRCC1 complex is the instability of Polβ, with no apparent impact on DNA repair. An earlier study had found that excess Polβ is ubiquitylated on the N terminus by the E3 ligases CHIP and MULE [30] , [31] . However, we found that proteasome-mediated degradation of free Polβ (not bound to XRCC1) is initiated by ubiquitylation on the C terminus, independent of CHIP or MULE. Here, we demonstrate that the scaffold protein XRCC1 also binds to and is regulated (stabilized) by the chaperone protein HSP90 when not bound to Polβ ( Figs 5b and 7c ). HSP90 is known to facilitate protein complex assembly [55] and the phosphorylated form (pHSP90) may be implicated in DNA repair complexes in response to DNA damage [51] . By binding and stabilizing XRCC1, we propose that pHSP90 promotes the formation of additional XRCC1 complexes (independent of Polβ). This depends on the cellular context such as proliferation status or damage response. In the absence of HSP90 (or following HSP90 inhibition), free XRCC1 (when not bound to Polβ or HSP90 or with other proteins) is removed by CHIP-mediated degradation. However, we find evidence for redundancy, suggestive of an as yet undetermined CHIP-independent mechanism of XRCC1 degradation. Whereas both proteins play a significant role in BER, they appear to function together in some aspects of BER, yet appear to have separate roles in others. Polβ-dependent BER predominates in the response to alkylating agents such as MNNG [56] ( Fig. 7a ). Due to the varied and different lesions induced by agents such as IR, H 2 O 2 or cis -Pt, the cellular response would likely require XRCC1-mediated repair that is both Polβ dependent and/or Polβ independent. XRCC1 availability and involvement is not only crucial in BER sub-pathways but also in other repair processes such as non-homologous end joining (NHEJ) or nucleotide excision repair (NER) [3] , [57] , [58] , [59] . Importantly, it has not been determined how cells regulate the Polβ/XRCC1 heterodimer nor the role for XRCC1 independent from Polβ. Within our proposed model, the repair protein complex architecture for the regulation of such DNA repair processes and in particular of BER sub-pathway choice is comprised of the archetype BER complex (Polβ/XRCC1), the stabilized XRCC1/(p)HSP90 complex and XRCC1* ( Fig. 7d ). Consistent with this model, complex formation (Polβ/XRCC1 versus XRCC1/HSP90) varies in response to DNA damage or cell proliferation status ( Fig. 7c ). We can speculate that the XRCC1/HSP90 or XRCC1/pHSP90 complexes might promote a role for XRCC1 in double-strand break repair [58] . Also, given that cis -Pt treatment results in more pHSP90/XRCC1 complex formation than following treatment with MNNG or H 2 O 2 , we might also speculate that this complex may play a role in NER. Such a role helps to explain why the level of XRCC1 is related to the resistance of cells to cis -Pt [60] . The ubiquitylation processes and pHSP90 binding revealed in this study provide the dynamics required for context-specific cellular response. This is particularly relevant in proliferating cells where the dynamics of the XRCC1/HSP90 complex is most pronounced in response to DNA damage ( Fig. 7c ). This is in line with earlier reports demonstrating that the level of Polβ determines radiation repair and survival in a proliferation-dependent manner [46] , [47] . We propose a dynamic model for the regulation of BER sub-pathway choice comprised of the archetype BER complex (Polβ/XRCC1), the stabilized XRCC1/pHSP90 complex and XRCC1* ( Fig. 7d ). Here we show that protein stability impacts BER protein complex formation, regulated by cell cycle and in response to DNA damage. We propose, in deference to earlier models, that DNA repair protein complexes can function as a regulatory mechanism governing protein stability. We suggest that the formation of the Polβ/XRCC1 and XRCC1/pHSP90 heterodimers regulate DNA repair pathway choice. Overall, these studies support a novel functional component of BER that may facilitate BER sub-pathway choice in response to DNA damage and cellular proliferation. We suggest that the pHSP90 and proteasome-mediated regulation of Polβ and XRCC1 is a universal mechanism of DNA repair pathway choice that is likely to respond to cell type, cell cycle and exogenous stimuli. Chemicals and reagents MEM, heat-inactivated fetal bovine serum (FBS), L -glutamine, antibiotic/antimycotic, geneticin, precast 4–20% Tris-glycine polyacrylamide gels and CyQuant GR reagent were from Invitrogen (Carlsbad, CA). Puromycin was from Clontech Laboratories. Gentamycin, cycloheximide (prepared as a 100 mM stock solution in ddH 2 O), N -ethylmaleimide (prepared as a 0.4 M stock solution in ethanol), Anti-Flag M2 affinity gel, 3 × Flag peptide, MG132 (prepared as a 10 mM stock solution in dimethylsulphoxide (DMSO)), 30% hydrogen peroxide solution and phenylmethanesulfonyl fluoride solution were from Sigma (St Louis, MO). Alpha EMEM was from MediaTech (Manassas, VA). MNNG (prepared as a 10 mM stock solution in DMSO) was from TCI America (# N0527; Portland, OR). 17-AAG (prepared as a 1 mM stock solution in DMSO) was from Tocris Bioscience (Park Ellisville, MO). Restore western blot stripping buffer, Pierce IP lysis buffer and RIPA buffer were from Thermo Scientific (Rockford, IL). DMSO was from Fisher Biotech (Fair lawn, NJ). Fugene 6 transfection reagent and protease inhibitor cocktail tablets were from Roche (Indianapolis, IN). The hybridoma cell clone #12CA5, expressing the anti-HA monoclonal antibody, was a generous gift from Kara Bernstein (Columbia University). The 12CA5 hybridoma cells were used to generate ascites and the resulting antibody was purified using protein-A-agarose and isotyped (IgG2b/kappa). Finally, the anti-HA antibody was linked to agarose for the IP studies described here. The ascites generation, protein-A purification, isotyping and linkage to agarose were all performed at Rockland Immunochemicals (Gilbertsville, PA). The hybridoma cell clone #10H, expressing the anti-PAR monoclonal antibody, was a generous gift from Matthias Ziegler (University of Bergen, Norway). The 10H hybridoma cells were used to generate ascites and the resulting antibody was purified using protein-A-agarose. The ascites generation and protein-A purification were performed at Rockland Immunochemicals. The hybridoma cell clone #18S, expressing the anti-Polβ monoclonal antibody, was a generous gift from Samuel H. Wilson (NIEHS, NIH). The 18S hybridoma cells were used to generate ascites and the resulting antibody was purified using protein-A-agarose. The ascites generation and protein-A purification were performed at Rockland Immunochemicals. The hybridoma cell clone #506-3D, expressing the anti-MPG monoclonal antibody, was a generous gift from Steve J. Kennel (ORNL). The 506-3D hybridoma cells were cultured and the antibody was purified using the Melon gel monoclonal IgG purification kit (Pierce). NucBuster protein extraction kit was from Novagen (San Diego, CA). MTS reagent (3-(4,5-dimethylthiazol-2-yl)-2, 5-diphenyltetrazolium bromide) was from Promega (Madison, WI). QuickChange XL Site-Directed Mutagenesis kit was from Stratagene (La Jolla, CA). All of the primers were synthesized and purified at Eurofins MWG/Operon. pBROAD3/TetR-KillerRed was made as described [61] . Lentiviral vectors for expression of Polβ and mutants Human Flag WT Polβ complementary DNA was PCR amplified and cloned into the pENTR/D-TOPO plasmid to create the pENTR-Flag-Polβ(WT) vector via a standard Topo-cloning methodology [18] . With this plasmid as template, residues K41, K61, K81, K206, K244, L301, V303 and V306 were mutated with the QuickChange XL Site-Directed Mutagenesis kit. The sequence of each primer is listed in Supplementary Table 1 . Briefly, we made the L301R, V303R and V306R mutations using primer pairs POLBL301R-F/POLBL301R-F, POLBV303R-F/POLBV303R-R and POLBV306R-F/POLBV306R-R, respectively. With the pENTR-Flag-Polβ(V306R) plasmid as template, we made the L301R/V306R and V303R/V306R mutations using primer pairs POLBL301R-F-6/POLBL301R-R-6 and POLBV303R-F-6/POLBV303R-R-6, respectively. With the pENTR-Flag-Polβ(L301R) plasmid as template, we made the L301R/V303R mutation using primers POLBL301R-F-3/POLBL301R-R-3. With the pENTR-Flag-Polβ(V303R/V306R) plasmid as template, the L301R/V303R/V306R (TM) mutation was constructed with primers POLBL301R-F-3-6/POLBL301R-R-3-6. A similar iterative strategy was used to develop the Flag-Polβ mutants K41R, K61R, K81R, K41R/K61R/K81R (KTM), K206A, K244A and K206A/K244A, as well as engineering the same mutants in the pENTR-Flag-Polβ(TM) vector (L301R/V303R/V306R). The vector pENTR-Flag-Polβ(K72A) was constructed as described previously [16] . Once sequence verified, the open-reading frames from each of the plasmids pENTR-Flag-Polβ(WT), pENTR-Flag-Polβ(L301R), pENTR-Flag-Polβ(V303R), pENTR-Flag-Polβ(V306R), pENTR-Flag-Polβ(L301R/V303R), pENTR-Flag-Polβ(L301R/V306R), pENTR-Flag-Polβ(L301R/V303R/V306R), pENTR-Flag-Polβ(K72A), pENTR-Flag-Polβ(KTM), pENTR-Flag-Polβ(TM/KTM), pENTR-Flag-Polβ(K206A), pENTR-Flag-Polβ(K244A), pENTR-Flag-Polβ(K206A/K244A), pENTR-Flag-Polβ(K206A/TM), pENTR-Flag-Polβ(K244A/TM), pENTR-Flag-Polβ(K206A/K244A/TM) and pENTR-EGFP were transferred into a Gateway-modified pLVX-IRES-puro vector, pLVX-IRES-Neo vector or pLVX-IRES-Hygro vector (Clontech) by TOPO cloning [16] . Positive clones were selected and plasmids were extracted with the QIAprep Spin Miniprep Kit (Qiagen). All the vectors developed and used in this study are listed in Supplementary Table 4 . Cell culture and cell line development All the cell lines developed and used in this study and their growth medium are listed in Supplementary Tables 2 and 3 . LN428 is an established glioblastoma-derived cell line with mutations in p53, deletions in p14ARF and p16, and is WT for PTEN [62] , [63] and is deficient in the expression of MGMT due to promoter methylation, as we have described [16] , [17] . LN428 glioblastoma cells, described previously [17] , were cultured in alpha MEM supplemented with 10% heat-inactivated FBS, L -glutamine, antibiotic/antimytotic and gentamycin. T98G cells were obtained from ATCC (Manassas, VA) and were cultured in MEM supplemented with 10% FBS, antibiotic/antimytotic, gentamycin, sodium pyruvate and MEM non-essential amino acids [64] . 88TAg and 92TAg cells were cultured in D-MEM high-glucose medium supplemented with 10% FBS, penicillin/streptomycin and glutamax [41] . The U2OS-TRE cell line was described previously as U2OS SCE 19 (ref. 65 ). In this cell line, 200 copies of a pTRE/I-SceI cassette is integrated in U2OS cells at a single integration site adjacent to the centromere of the X chromosome [26] . Cell lines were developed by lentiviral transduction and stable integration selection. Lentiviral particles were generated by co-transfection of four plasmids (control plasmid (pLVX-EGFP-IRES-puro, pLVX-EGFP-IRES-neo or pLVX-EGFP-IRES-hygro) or pLVX-Flag-Polβ(WT)-IRES-puro (or neo) (or Polβ mutants) together with pMD2.g(VSVG), pVSV-REV and pMDLg/pRRE) into 293-FT cells using FuGene 6 Transfection reagent. Forty-eight hours after transfection, lentivirus-containing supernatant was collected and passed through 0.45 μM filters to isolate the viral particles. Lentiviral transduction was performed as follows: cells (6 × 10 4 ) were seeded into a six-well plate 24 h before transduction. Lentiviral particles were mixed with polybrene (2 μg ml −1 ) and then added to the cells, incubating at 32 °C overnight. Cells were then cultured for 72 h at 37 °C and were then selected by culturing in selection medium for 1–2 week(s). In most cases, cells transduced with an EGFP-expressing lentivirus were used as control. Where indicated, cells were depleted of endogenous Polβ by shRNA-mediated RNA interference (LN428/Polβ-KD), specific for the Polβ 3′UTR to allow re-expression of the Flag-tagged recombinant proteins [16] , [17] , [18] , [66] . Using this knockdown/re-expression system, similar stable cell lines were developed by transduction of LN428/MPG/Polβ-KD, T98G and T98G/MPG/Polβ-KD cells as will be described throughout the text (see Supplementary Tables 2 and 3 ). Briefly, LN428 cells overexpressing MPG (LN428/MPG), LN428/MPG cells deficient in Polβ (LN428/MPG/Polβ-KD), LN428 cells deficient in XRCC1 (LN428/XRCC1-KD) and T98G/MPG cells deficient in Polβ (T98G/MPG/Polβ-KD) were established previously [16] , [67] . LN428 cells expressing Flag-Polβ(WT) and Polβ mutants including L301R, V303R, V306R, L301RV303R, L301RV306R, TM and K72A, LN428/MPG/Polβ-KD cells expressing Flag-Polβ(WT) and Flag-Polβ mutants including Flag-Polβ(TM) and Flag-Polβ(K72A), LN428/XRCC1-KD cells expressing Flag-Polβ(WT) and Flag-Polβ(TM), T98G cells expressing Flag-Polβ(WT) and Flag-Polβ(TM) and T98G/MPG/Polβ-KD cells expressing Flag-Polβ(WT) and Flag-Polβ mutants including Flag-Polβ(L301R/V303R) or Flag-Polβ(TM) were developed as follows: [16] lentiviral particles were generated by co-transfection of four plasmids (control plasmid (pLVX-EGFP-IRES-puro, pLVX-EGFP-IRES-neo or pLVX-EGFP-IRES-hygro) or pLVX-Flag-Polβ(WT)-IRES-puro (or neo) (or Polβ mutants) together with pMD2.g(VSVG), pVSV-REV and pMDLg/pRRE) into 293-FT cells using FuGene 6 Transfection reagent. Forty-eight hours after transfection, lentivirus-containing supernatant was collected and passed through 0.45 μM filters to isolate the viral particles. Lentiviral transduction was performed as follows: cells (6 × 10 4 ) were seeded into a six-well plate 24 h before transduction. Lentiviral particles were mixed with polybrene (2 μg ml −1 ) and then added to the cells, incubating at 32 °C overnight. Cells were then cultured for 72 h at 37 °C and were then selected by culturing in selection medium for 1–2 week(s). Nuclear extracts (20–30 μg) were analysed by immunoblotting to determine the expression of the desired proteins. All cells were cultured at 5% CO 2 and 37 °C, except MEFs, including 88TAg and 92TAg, which were cultured at 10% CO 2 . IP and immunoblot For newly developed stable cell lines, the expression level of proteins was determined by immunoblot using nuclear lysates. Nuclear lysates were prepared with NucBuster protein extraction kit, and protein concentration was determined with the Bio-Rad protein assay dye reagent (Bio-Rad). For the PAR assay, Polβ and XRCC1 stability assay, CHIP-mediated degradation of XRCC1 and the degradation of BER proteins induced by HSP90 knockdown, whole-cell lysates (WCLs) were used for the immunoblot. To prepare WCLs, 2–2.5 × 10 5 cells were seeded into a 60-mm cell culture dish. Twenty-four hours later, cells were treated with different drugs (as needed, using conditions described in the figure legends), cells were washed twice with cold phosphate-buffered saline (PBS), then cells were collected and lysed with 80 μl of 2 × clear Laemmli buffer (2% SDS, 20% glycerol, 62.5 mmol l −1 Tris-Hcl, pH 6.8). Cell lysates were boiled for 8 min and quantified using a DC protein assay following the microplate protocol provided by the company with the DC protein assay kit (Bio-Rad). To study the interaction of Polβ and XRCC1, anti-Flag M2 affinity gel was used to immunoprecipitate Flag-Polβ(WT) and Flag-Polβ mutants. Cells from 2 × 150 mm dishes (70–90% confluent) were collected and lysed in 1 ml of Pierce IP lysis buffer with protease inhibitor. The anti-Flag M2 affinity gel was prepared according to the protocol provided by the company. Briefly, the gel was washed three times with 5 × bead volume of 0.1 M glycine, pH 3.5, three times with 5 × bead volume of Tris-buffered saline (TBS) buffer (50 mM Tris-HCl, pH 7.4, 150 mM NaCl) and twice with 5 × bead volume of IP lysis buffer. The gel was suspended in 150 μl of IP lysis buffer with protease inhibitor and mixed with 1 ml cell lysate. The mixture was shaken overnight at 4 °C. Next day, the mixture was centrifuged to pellet the gel and the supernatant was removed. Then, the gel was washed five times with 1 ml IP lysis buffer and three times with 1 ml TBS buffer containing protease inhibitor. Finally, proteins bound to the gel were eluted with 200 μl of Flag peptide elution buffer (200 μg ml −1 3 × Flag peptide in TBS buffer with protease inhibitor) twice and with 200 μl TBS buffer once. The eluted product was collected and concentrated with Amicon Ultra-2ml 3k centrifugal filters (Millipore). The immunoprecipitated proteins were quantified as above. To study the interaction of HSP90 with XRCC1 and Polβ, anti-HA (clone 12CA5) agarose was used to pull down HA-HSP90 and binding proteins. The cell lysis and agarose preparation, binding and washing were performed as described above. In the elution step, 35 μl of 2 × Laemmli buffer was added to the agarose and boiled 5 min. The mixture was centrifuged to pellet the agarose and the supernatant was collected. To study the interaction of endogenous HSP90 with XRCC1 or other BER-related proteins, HSP90 antibody (1:1,000; AC88, Abcam) and XRCC1 antibody (1:4,000; A300-065A, Bethyl Labs) were used to pull down HSP90 or XRCC1 and bound proteins were analysed by immunoblot. To study the ubiquitylation of Polβ and XRCC1 in cells and the dynamic interaction of Polβ and HSP90 with XRCC1, IP was performed with the corresponding primary antibody and protein G. The detailed procedures can be found in the manual provided by Santa Cruz Technology. For immunoblot, 20–30 μg nuclear extract or 8–15 μg WCL or 0.2–0.5 μg immunoprecipitated proteins were loaded on a precast 4–12% NuPAGE Tris-glycine gel, run 2–3 h at 100 V. The gel was transferred to a 0.45-μm nitrocellulose membrane (Bio-Rad) at 0.2 mA for 2–3 h. The membrane was blotted with primary antibodies. The following primary antibodies were used: anti-PARP1 (1:1,000; BD Pharmingen), anti-XRCC1 (1:4,000; Bethyl Labs), anti-XRCC1 (1:500; 33-2-5, Abcam), anti-Polβ (1:1,000; Clone 61; Thermo Scientific or 1:5,000; Clone 18S), anti-MPG (1:1,000; Clone 506-3D), anti-PCNA (1:2,000; SC-56; Santa Cruz Biotechnology), anti-APE1 (1:5,000; NB 100-16; Novus Biologicals), anti-MGMT (1:1,000; NB100-168; Novus Biologicals), anti-PAR (1:1,000; Clone 10H), anti-HA (1:5,000; Clone 12CA5), anti-OGG1 (1:250; NB100-106; Novus Biologicals), anti-Flag (1:1,000; M2, Sigma), anti-HSP90 (1:1,000; S88, Novus Biologicals) and anti-phospho-HSP90α (Thr5/7) (1:1,000; Cell Signalling). After washing, secondary antibodies were used to blot the membrane. The following secondary antibodies were used: Immun-Star Goat anti-mouse-HRP conjugate (1:5,000; Bio-Rad) and Immun-Star Goat anti-rabbit-HRP conjugate (1:5,000; Bio-Rad). After washing, the membrane was illuminated with Immun-Star HRP peroxide buffer with luminol/enhancer (Bio-Rad). If no signal can be detected, then membrane was illuminated with SuperSignal west femto maximum sensitivity substrate (Thermo Scientific). If necessary, protein bands were quantified by Image J. Uncropped immunoblots are provided in Supplementary Figs 9 and 10 . Cytotoxicity assay H 2 O 2 - and MNNG-induced cytotoxicity was determined by both short-term (MTS) and long-term (CyQuant) cytotoxicity assays. Short-term (48 h) cytotoxicity was evaluated by an MTS assay and long-term (10 day) cytotoxicity was evaluated by a CyQuant assay. Results were calculated from the average of three or four separate experiments and reported as the percent survival compared with the cells without drug treatment. For the MTS assay, LN428 cells were seeded 24 h before treatment at 2,000 cells per well in 96-well plates. For H 2 O 2 -induced cytotoxicity, LN428/EGFP (control), LN428/Polβ(K72A), LN428/Polβ(WT) and LN428/Polβ(TM) cells were treated with freshly prepared H 2 O 2 (0, 60, 100, 120, 140, 160 or 180 μM) in selection media for 48 h. For MNNG-induced cytotoxicity, LN428/MPG/Polβ-KD/EGFP, LN428/MPG/Polβ-KD/Polβ(WT), LN428/MPG/Polβ-KD/Polβ(TM) and LN428/MPG/Polβ-KD/Polβ(K72A) cells were treated with freshly prepared MNNG (0, 1, 2, 3, 4, 5 or 6 μM) in selection media for 48 h. After removing the medium, cells were incubated with CellTiter solution (Promega, G356B) for 3 h at 37 °C. The absorbance at 490 nm was measured in a microplate reader. Cell survival was calculated as the ratio of the absorbance for cells treated with drug as compared with cells without drug treatment. H 2 O 2 - and MNNG-induced long-term cytotoxicity was evaluated using the CyQuant assay [20] . For H 2 O 2 -induced cytotoxicity, cells from LN428/EGFP, LN428/Polβ(K72A), LN428/Polβ(WT) and LN428/Polβ(TM) cell lines were seeded at 60 cells per well in 96-well plates. For MNNG-induced cytotoxicity, cells from T98G/MPG/Polβ-KD/EGFP, T98G/MPG/Polβ-KD/Polβ(WT), T98G/MPG/Polβ-KD/Polβ(L301RV303R) and T98G/MPG/Polβ-KD/Polβ(TM) cell lines were seeded at 80 cells per well in 96-well plates. After 24 h, cells were treated with freshly prepared H 2 O 2 (0, 10, 20, 30, 40, 50, 60 or 70 μM) in selection media or freshly prepared MNNG (0, 0.2, 0.5, 0.8, 1 or 2 μM) in selection media. Cells were incubated 8–10 days without removal of the drug. The following steps were the performed according to the manufacturer’s instructions. Briefly, cells were washed with PBS. After the complete removal of PBS, the microtiter plates were sealed with parafilm and frozen at −80 °C overnight. Next day, 200 μl of cell lysis solution with CyQuant dye was added to each well. The plates were sealed with Parafilm and covered with aluminium foil to keep plates from the light and shaken for 1 h at room temperature, then incubated overnight in the freezer (−30 °C). Next day plates were taken out from the freezer and thawed slowly at room temperature. Finally, plates were read on a fluorescent plate reader. Results were calculated from the average of three or four separate experiments and reported as the percent survival compared with the cells without drug treatment. An untreated control in which only 50% of the cells were seeded is always included to ensure linearity of the assay. Lentiviral transduction and plasmid transfection Lentiviral particles were generated by co-transfection of four plasmids (the shuttle vector plus three packaging plasmids: pMD2.g(VSVG), pVSV-REV and PMDLg/pRRE) into 293-FT cells using FuGene 6 Transfection Reagent (Roche). Forty-eight hours after transfection, lentivirus-containing supernatant was collected and passed through 0.45 μM filters to isolate the viral particles. Lentiviral transduction was performed as follows: cells (6 × 10 4 ) were seeded into a six-well plate 24 h before transduction. Lentiviral particles were mixed with polybrene (2 μg ml −1 ) and then added to the cells, incubating at 32 °C overnight. Cells were cultured for 72 h at 37 °C and were then selected by culturing in growth media with 1.0 μg ml −1 puromycin. For plasmid vectors including pcDNA-HA-HSP90, pCMVTags-Flag-CHIP, pcDNA-HA-ubiquitin, pDsRed-RFP-XRCC1 and pRS1427 (31 kDa C-terminal domain of Polβ), transient transfection was carried out with FuGene 6 Transfection Reagent according to the manufacturer’s instruction. Radiation sensitivity and clonogenic survival assay Radiation sensitivity was assessed by colony formation assay. Proliferating LN428 cells were plated with varying cell concentrations and irradiated after 16 h using the 137 Cs irradiation unit Gammacell-40 with a dose rate of 1.1 Gy min −1 at room temperature. Cells were allowed to grow for another 14 days to form colonies before rinsing in PBS, fixing in methanol and staining with 1% crystal violet. Colonies consisting of 50 cells or more were counted by eye under an inverted dissecting microscope. Survival was calculated relative to the plating efficiency of un-irradiated controls. CopGFP-Polβ fusion and fluorescence imaging A copGFP-Polβ fusion plasmid was constructed using pCT-CMV-copGFP-MCS-EF1-puro (System Biosciences). Forward primer (PolBGFPC24F) and reverse primer (PolBGFPC24R) were designed as: PolBGFPC24F: 5′-CTGCCAGGGTCTAGAATGGACTACAAAGACGATGAC-3′ and PolBGFPC24R: 5′-CGCAGAGCCGGATCCTCATTCGCTCCGGTCCCTTGG-3′. The Polβ open-reading frame was PCR amplified to engineer the restriction enzyme sites XbaI and BamHI for cloning in-frame with copGFP using standard protocols. PCR was performed with pENTR-Flag-Polβ(WT) and pENTR-Polβ(TM) as template. After PCR, products were digested with XbaI and BamHI, purified fragments were ligated into the pCT-CMV-copGFP-MCS-EF1-puro lentiviral vector (System Biosciences, Mountain View, CA) hydrolysed by XbaI and BamHI. Positive colonies were selected and sequenced. Sequence-verified plasmids were transiently transfected and lentivirus production was as described above. For cell imaging analysis, LN428 and LN428/MPG cells were seeded on glass-bottom dishes for 24 h, then cells were transduced with the lentiviral vector expressing copGFP-Polβ(WT), copGFP-Polβ(TM) or copGFP (control) as described above. After 16–18 h, the media containing lentiviral particles were removed and cells were transiently transfected with pRFP-XRCC1 as described above. 48 h later, cells were treated with 5 μM MNNG and fluorescence images were obtained and processed using a FV-1000 confocal scanning laser microscopy system (Olympus, Tokyo). A laser system (405 nm; Photonic Instruments, St Charles, IL) coupled to the epifluorescence path of the microscope was also used to treat cells expressing RFP-XRCC1 and the copGFP fusion proteins. For the PARP inhibition assay, 4 μM PJ34, 10 μM ABT-888 and 5 μM BMN-673 were used to pre-treat cells for 1 h. The control fluorescence images were obtained. Then cells were exposed to 50 or 100 ms 405 nm laser light for different time courses and images were obtained. For the assay to examine the kinetics of recruitment of Polβ and whether PARP inhibitors block the recruitment of Polβ, the foci intensity was quantified by the Image J program. KillerRed and copGFP-Polβ(WT), copGFP-Polβ(TM) or copGFP (control) were expressed in U2OS-TRE cells (transient) as described above. Cells with or without 4 μM PJ34 treatment for 0.5–1 h were exposed to light and processed by using the FV-1000 confocal scanning laser microscopy system to obtain the fluorescent images and the foci intensity was quantified by the Image J program. Stability assays for Polβ and XRCC1 To study the stability of Polβ or Polβ mutants, the corresponding cells expressing the desired proteins were seeded and 24 h later, cells were treated with 0.2 mM cycloheximide (Cyclo) or 0.2 mM Cyclo plus 25 μM MG132. The time course for cells treated with drugs for 30 min was set as ‘0’. After cells were treated with drugs for the designed time course, drugs were removed and WCL was prepared and quantified as described above. The level of Polβ and XRCC1 was determined by immunoblot and the intensity of bands was quantified using the Image J program. The level of PCNA was set as a loading control. To study the stability of XRCC1, seeded cells were treated with different doses of 17-AAG for 24 h, then 17-AAG was removed and cells were treated with Cyclo or Cyclo plus MG132 as described above. WCL was prepared and the level of XRCC1 was determined and quantified. To study CHIP-mediated degradation of BER proteins, the seeded cells were set up in four groups: two of the four groups were transiently transfected with pCMVTag2-Flag-CHIP. After 48 h, cells from one non-transfected group and one transfected group were treated with 10 μM 17-AAG and the other two groups were treated with DMSO overnight. WCL was prepared and the level of XRCC1, Polβ, PCNA and CHIP was determined. qRT–PCR analysis Expression of Polβ and CHIP was measured by qRT–PCR using an Applied Biosystems StepOnePlus system [16] . Briefly, 80,000 cells were lysed and reverse transcribed using the Applied Biosystems Taqman Gene Expression Cells-to-CT kit. Analysis of mRNA expression was performed as per the instruction of the manufacturer (ΔΔ C T method) using Applied Biosystems TaqMan Gene Expression Assays: Hs00160263-m1 (human Polβ) and Hs01071598-g1 (CHIP). Samples were run in triplicate and the results shown are the mean±s.d. of all three analyses. Each are normalized to the expression of human β-actin (part #4333762T). Modulation of XRCC1 complexes with Polβ or HSP90 92TAg cells were seeded in a 60-mm dish or 150-mm dish and incubated for 48 h. Cells that were ~50% confluent were defined as proliferating cells, as confirmed by flow cytometry. Cells that were ~100% confluent were defined as confluent cells. Proliferating or confluent cells without drug treatment or treated with 5 μM MNNG, 150 μM H 2 O 2 , 5 μM cis -diamineplatinum(II) dichloride ( cis -Pt) or 3 Gy IR for different times were collected and WCL was prepared and used for the IP assay. The IP assay was performed with the XRCC1 antibody and protein G-plus agarose as described above. The level of pulled-down HSP90, pHSP90 or Polβ and input XRCC1 was determined by immunoblot with the corresponding antibody. The levels of XRCC1, HSP90, pHSP90 and Polβ in WCL were also determined. Cell cycle phase distribution of proliferating or confluent cells was determined by DNA content analysis with propidium iodide (Invitrogen) staining. Cells were trypsinized and fixed in 70% ice-cold ethanol for 30 min. The cells were then washed with 1%BSA/PBS buffer and permeabilized with 0.25% Triton X-100 in 1%BSA/PBS. Finally, cells were incubated in PBS containing propidium iodide (50 μg ml −1 ) and RNAse A (40 μg ml −1 ) [68] . The samples were analysed on a CyAn-ADP Analyzer (Beckman Coulter, Brea, CA). Data were analysed with Summit software. HSP90 and CHIP knockdown Lentiviral vectors expressing five shRNAs to knockdown HSP90 or CHIP were from Sigma and prepared by the UPCI Lentiviral Core Facility. The sequence of each shRNA is listed in Supplementary Table 1 . Lentiviral preparation and cell transduction are described above. Statistical analysis All data are shown as a mean±s.d. from three independent experiments. Student’s t -test was used for comparisons between two groups. For multiple comparisons, one-way analysis of variance was used. Statistical analysis was performed using GraphPad PRISM. Determination of ubiquitylated Pol β and XRCC1 in cells LN428/Polβ(TM), LN428/Polβ(TM/K206A/K244A) and T98G/Polβ(TM) cells were transiently transfected with pcDNA-HA-ubiquitin to express HA-ubiquitin. Forty-eight hours later, cells with or without HA-ubiquitin transfection were treated with 25 μM MG132 for 8 h. Cells were lysed with Pierce IP lysis buffer containing protease inhibitor and 5 mM N -ethylmaleimide (NEM). The supernatants of cell lysates were collected and incubated with M2 (5 μg) or XRCC1 (5 μg) antibody overnight and then incubated with protein G agarose for 4 h. For details, see above. The eluted IP products were probed with HA antibody. Liquid chromatography—tandem mass spectrometry analysis To determine the proteins bound to either WT Polβ or the mutant form (TM) of Polβ, WCLs were prepared from stable LN428-derived cell lines expressing GFP (Cont), the WT version of Polβ, Flag-Polβ(WT), or the mutant version of Polβ, Flag-Polβ(TM). The Flag-Polβ transgene (as well as the interacting proteins) was then bound to Flag-M2-agarose and the beads were extensively washed in cell lysis buffer (Pierce IP lysis buffer with protease inhibitor), as detailed above. Immunoprecipitated samples were separated by SDS–PAGE (Bolt 4–12% Bis-Tris Plus Gel, Life Technologies, Grand Island, NY) to about 1 cm (150 V for 10 min) and stained with Simply Blue SafeStain (Life Technologies). After washing with Milli-Q water, the whole stained regions were excised, washed with HPLC water and destained with 50% acetonitrile/25 mM ammonium bicarbonate until no visible blue staining. Gel pieces were dehydrated with 100% acetonitrile, reduced with 10 mM dithiothreitol (DTT) at 56 °C for 1 h, followed by alkylation with 55 mM iodoacetamide (IAA) at room temperature for 45 min in the dark. Gel pieces were then again dehydrated with 100% acetonitrile to remove excess DTT and IAA, and rehydrated with 20 ng μl −1 trypsin in 25 mM ammonium bicarbonate and digested overnight at 37 °C. The resulting tryptic peptides were extracted with 70% acetonitrile/5% formic acid, speed-vac dried and re-constituted in 18 μl 0.1% formic acid. One μl of extracted tryptic peptides for each sample was analysed with reverse-phased liquid chromatography–tandem mass spectrometry (LC–MS/MS) using a nanoflow LC (EASY-nLC II, Thermo Scientific, San Jose, CA) coupled online to LTQ/Orbitrap Velos Elite hybrid mass spectrometer (Thermo-Fisher, San Jose, CA). Solvent A (0.1% formic acid in HPLC grade water) and solvent B (0.1% formic acid in 100% acetonitrile) were used as the mobile phase. Peptides were first loaded onto a 20-μl capillary sample trap column (Thermo Scientific, San Jose, CA) and desalted on-line for 6 μl solvent A. Peptides were then eluted onto a capillary column (75 μm inner diameter × 360 μm outer diameter × 15 cm long; Polymicro Technologies, Phoenix, AZ) slurry-packed-in-house with 5 μm particle size, 125 Å pore size C-18 silica-bonded stationary phase (Phenomenex, Torrance, CA) and resolved using a 100-min gradient at the flow rate of 0.2 μl min −1 (3–33% B for 90 min, 33–80% B for 2 min, constant at 80% B for 6 min and then 80–0% B for 2 min). Eluted peptides were analysed via electrospray ionization to the mass spectrometer. Data were collected in positive ionization mode, with FT MS1 AGC targets=100,000, maximum injection time=200 ms, spray voltage=2.5 kV and capillary temperature=325 °C. Acquisition consisted of a cycle of a full-scan FT mass spectrum at a resolution of 60,000 and top 20 MS/MS spectra recorded sequentially on the most abundant ions on the ion trap. MS/MS spectra were searched by COMET against an indexed human database build from a non-redundant NCBI human database with the following modifications: static modification of cysteine (carboxyamidomethylation, +57.02 Da) and variable modification of methionine (oxidation, +15.99 Da). The mass tolerance was set to 20 p.p.m. for precursor ions and 0.8 Da for fragment ions. The raw data was organized in a three by nine factorial design (that is, three conditions, each having nine biological replicates). Custom software (dMS 1.0, University of Pittsburgh and InfoClinika) was used to align and integrate the XRCC1-extracted ion chromatograms for the Cont, WT and TM samples. Relative quantitation is achieved by comparing the sum of all isotopes of particular defined peptides. Each resulting feature is defined by its particular m / z , elution time, charge state and intensity. How to cite this article: Fang, Q. et al. HSP90 regulates DNA repair via the interaction between XRCC1 and DNA polymerase β. Nat. Commun. 5:5513 doi: 10.1038/ncomms6513 (2014).